A signal cascade originated from epidermis defines apical-basal patterning of Arabidopsis shoot apical meristems In multicellular organisms, a long-standing question is how spatial patterns of distinct cell types are initiated and maintained during continuous cell division and proliferation. Along the vertical axis of plant shoot apical meristems (SAMs), stem cells are located at the top while cells specifying the stem cells are located more basally, forming a robust apical-basal pattern. We previously found that in Arabidopsis SAMs, the HAIRY MERISTEM (HAM) family transcription factors form a concentration gradient from the epidermis to the interior cell layers, and this gradient is essential for the stem cell specification and the apical-basal patterning of the SAMs. Here, we uncover that epidermis specific transcription factors, ARABIDOPSIS THALIANA MERISTEM LAYER 1 (ATML1) and its close homolog, define the concentration gradient of HAM in the SAM through activating a group of microRNAs. This study provides a molecular framework linking the epidermis-derived signal to the stem cell homeostasis in plants. Plant shoot apical meristems (SAMs) is the sustainable resource for the shoot and flower development [1] . In the model plant Arabidopsis, several key pathways in control of stem cell homeostasis in the SAMs have been identified [2] , [3] , [4] . Among them, the HAIRY MERISTEM (HAM) family GRAS ( G AI, R G A and S CR) domain transcription factors play essential roles in determining the specification and proliferation of stem cells in the SAMs [4] , [5] , [6] , [7] , [8] , [9] . Two HAM family members, HAM1 and HAM2 proteins, interact with the homeodomain transcription factor WUSCHEL (WUS) and function together with WUS to regulate downstream gene expression and maintain the stem cell homeostasis [7] , [8] . In addition, HAM1 and HAM2 keep the CLV3 expression off at the inner cell layers to establish an apical-basal polarity of the SAMs and the de novo axillary stem cell niches [9] , [10] . Through both computational modeling and experimentation, we previously found that HAM1/2 are expressed with a concentration gradient from the epidermis to the deep cell layers in the SAMs, which is important for the stem cell homeostasis in the established SAM [9] . In the de novo formation of axillary meristems, this HAM gradient is formed from early to late developmental stages and it is essential for the patterning of newly initiated stem cell niches. However, how this concentration gradient of HAM is defined in the developing meristem and continually maintained in the established SAMs remains to be elucidated. The conserved microRNA171 (miR171) family in Arabidopsis has been reported to specifically repress the HAM family genes [11] , [12] , [13] . miR171, the 21-ribonuleotide species, specifically recognizes and cleaves HAM1 , HAM2 , and HAM3 [11] , [12] . miR171 originates from the products of four genes in Arabidopsis including MIR171A , MIR171B , MIR171C , and MIR170 [14] , [15] , [16] . Several studies have reported that miR171 is expressed in a wide range of tissues including cotyledons, hypocotyls, leaves, meristems, and flowers [11] , [12] , [17] , [18] . One recent study reported that MIR171A , one of MIR171 genes, is expressed in the epidermal layer during the embryogenesis and vegetative development stages [19] . In this work, we establish a molecular linkage between the epidermis specific transcription factors, including ARABIDOPSIS THALIANA MERISTEM LAYER 1 (ATML1) and its close homolog PROTODERMAL FACTOR 2 (PDF2) [20] , [21] , [22] , [23] , [24] , [25] , [26] , [27] , [28] , and the expression of MIR171 . Combining in vitro biochemistry, in vivo live imaging, and in silico modeling approaches, we uncover the mechanism underlying how the epidermis expressed ATML1/PDF2 patterns the concentration gradient of HAM via miR171 in the established SAMs and de novo initiating stem cell niches. MIR171/170 are specifically expressed in the SAM epidermis To define and compare the expression patterns of three MIR171 genes and one MIR170 gene in the SAMs, we generated transcriptional reporters for these genes in which a fluorescent protein is placed in between their own 5′ promoters and 3′ terminators (Fig. 1a–d ). Through the confocal live imaging of the SAMs using identical settings, surprisingly, we found that in the SAMs and the floral meristems (FMs), the expressions of all four reporters are restricted to the epidermis. In the SAMs, MIR171A and MIR171B ( pMIR171A::H2B-GFP and pMIR171B::H2B-GFP ) are expressed at high levels (Fig. 1a (panels 1–3), Fig. 1b (panels 1–3)) (Supplementary Movies 1 and 2 ), while MIR171C and MIR170 ( pMIR171C::H2B-GFP and pMIR170::H2B-GFP ) are expressed at very low levels (Fig. 1c (panels 1–3), Fig. 1d (panels 1–3)) (Supplementary Movies 3 and 4 ). In the young seedlings, pMIR171A::H2B-GFP and pMIR171B::H2B-GFP are also specifically expressed in the epidermis of the developing leaves and hypocotyls (Fig. 1a (panels 4–5), Fig. 1b (panels 4–5). In contrast, the pMIR171C::H2B-GFP reporter activity is undetectable from young leaves and hypocotyl in the seedling, and pMIR170::H2B-GFP is weakly expressed in the developing young leaves and hypocotyls (Fig. 1c (panels 4–5), Fig. 1d (panels 4–5)). These results showed that similar to MIR171A [19] , MIR171B expression is strongly activated and specifically confined in the epidermal layer, whereas, the expression of MIR171C and MIR170 is also specifically restricted at epidermis of the SAM but their expression level is very low (Fig. 1a–d ). Fig. 1: Epidermis expressed MI R 170/171 genes define the apical-basal gradient of HAM in Arabidopsis SAMs. a The pMIR171A::H2B-GFP reporter is highly expressed at the epidermis in the SAM (panels 1–3) and in the young leaves (panels 4–5). b The pMIR171B::H2B-GFP reporter is highly expressed at the epidermis in the SAM (panels 1–3) and in the young leaves (panels 4–5). c The pMIR171C::H2B-GFP reporter is weakly expressed at the epidermis in the SAM (panels 1–3) and undetectable in the young leaves (panels 4–5). d The pMIR170::H2B-GFP reporter is weakly expressed at the epidermis in the SAM (panels 1–3) and in the young leaves (panels 4–5). e The pHAM2::YPET-HAM2 reporter that is sensitive to the miR170/171 is expressed with a concentration gradient in the SAM, with high expression at inner cell layers and no expression in epidermis (panels 1–3). The pHAM2::YPET-HAM2 reporter is not expressed at the epidermis of the young leaves (panels 4–5). f The pHAM2::H2B-GFP reporter that is not sensitive to miR170/171 is highly expressed in all the cell layers (including the epidermal layer) in the SAM (panels 1–3), and the pHAM2::H2B-GFP reporter is highly expressed at the epidermis of the young leaves (panels 4–5). Panels (from left to right): 1, orthogonal view of a SAM; 2, transverse section view of L1 in the SAM; 3, transverse section view of corpus in the SAM; 4, section view of a seedling; 5, 3D projection view of the seedling. Channels: GFP/YFP (green), propidium iodide (PI) counterstain (purple), and Chlorophyll (red). Scale bar: (panels 1–3) 20 µm; (panels 4–5) 100 µm. Full size image In addition, consistent with our previous report [9] , the HAM2 translational reporter pHAM2::YFP-HAM2 in ham123 showed a concentration gradient in the SAM (Fig. 1e ) (Supplementary Movie 5 ). However, the HAM2 transcriptional reporter pHAM2::H2B-GFP , which lacks the miR171 binding site, is highly expressed in all cell layers of the SAM (Fig. 1f ) (Supplementary Movie 6 ). These results suggest that miR171 keeps HAM off in the L1 layer and it further shapes the HAM gradient, likely through the movement from L1 to L2 or even upper layers of the corpus to suppress HAM. Epidermis specific ATML1/PDF2 directly upregulate MIR171A/B The expression patterns of the MIR171A and MIR171B reporters in epidermis of the SAMs (Fig. 1a , b) are almost identical to that of the ATML1 and PDF2 [20] , [21] , which are epidermis specific transcription factors. Thus, we decided to examine whether these two genes are directly regulated by ATML1 and PDF2. First, we tested the interaction between ATML1 or PDF2 protein and the promoter DNA of MIR171A using the yeast one hybrid (Y1H) system (Fig. 2a, b ). Both the β-galactosidase liquid and x-gal lifting assays showed that ATML1 and PDF2 proteins interact with the full-length promoter of MIR171A (Fig. 2a, b , Supplementary Fig. 1a ). Because ATML1/PDF2 was reported to bind to an L1 box motif [22] , [29] , we searched along the MIR171A promoter for putative ATML1/PDF 2 binding sites. We used the conserved DNA sequences from the previously reported L1-box motifs [22] , [29] to perform the search and we identified three regions that contain the conserved TT(A/T)AATG(C/T) sequences (Fig. 2a ). We then generated new reporters for Y1H assays, each of which contains a fragment of the MIR171A promoter DNA that includes one putative L1 box (Fig. 2a, c–e ). The Y1H assays showed that all three fragments (F1, F2 and F3) interact with both ATML1 and PDF2 (Fig. 2c–e ). We further confirmed these protein-DNA interactions by the electrophoresis mobility shift assays (EMSA). We labeled these DNA fragments with Cy5 (Fig. 2a ), and when each of the Cy5-labeled probe was incubated with recombinant GST ATML1 30–134 , the DNA binding domain of the ATML1 (Supplementary Fig. 2 ), the Cy5-labeled DNA probe with reduced gel mobility representing the protein-DNA complex was observed in the native gel (Fig. 2f–k ). This shifted band was not observed when GST was incubated with the Cy5-labeled probe (Fig. 2f, h, j ), nor when excess amount of additional unlabeled probe (competitor) was supplied prior to the incubation with GST ATML1 30–134 (Fig. 2g, i, k ), demonstrating the specificity of the interaction in EMSA. We further examined whether MIR171A can be directly regulated by ATML1 using a dual-luciferase reporter assay. Compared to empty vector controls, the expression of the pMIR171A::LUC reporter is significantly induced by the ATML1 effector in the tobacco transient expression system (Fig. 2l ). Fig. 2: ATML1 and PDF2 directly activate MIR171A . a Schematic structure of the MIR171A promoter. The expanded diagram shows the sequences of putative L1 boxes on the promoter. Probes indicate the DNA fragments used in the EMSA and the yeast one hybrid (Y1H) assay, and +1 indicates the transcription start site. b The full-length promoter of MIR171A interacts with ATML1 and PDF2 proteins in Y1H assays. Y-axis: the relative activity of the pMIR171A:: lacZ reporter. All the numbers are normalized to the average value of the empty vector control. Bars: mean ± standard error (SE) ( n = 3 biological replicates). ** P < 0.01, *** P < 0.001 (Student’s two-tailed t -test). c – e Different DNA fragments from the MIR171A promoter interact with ATML1 and PDF2 proteins in Y1H. Y-axis: the relative activity of the pMIR171A-F1::lacZ ( c ), pMIR171A-F2::lacZ ( d ) and pMIR171A-F3:: lacZ ( e ) reporters. All the numbers are normalized to the average value of the empty vector control. Bars: mean ± SE ( n = 5 biological replicates). ** P < 0.01, *** P < 0.001 (Student’s two-tailed t -test). f – k Electrophoretic mobility shift assay (EMSA) shows that GST ATML1 30–134 but not GST binds to the Cy5-labeled probes including MIR171A-F1 ( f ), MIR171A-F2 ( h ) and MIR171A-F3 ( j ). The GST ATML1 30–134 –induced mobility shift of the Cy5-labeled DNA probe can be chased away when excess amount of the unlabeled DNA probe (chase) is present ( g , i , k ). Arrows indicate free DNA probes and DNA-protein complexes. l Dual-luciferase assays show that ATML1 activates the transcription of MIR171A . Left panel: structure of the reporter construct. Term, CaMV terminator; LB, transfer DNA (T-DNA) left border; RB, T-DNA right border. Right panel: LUC/REN, ratio of firefly luciferase (LUC) to Renilla luciferase (REN) activity. The LUC/REN in tobacco cells co-transformed with the reporter pMIR171A::LUC and the ATML1 effector ( n = 9 biological replicates) is significantly higher than that in the cells co-transformed with the same reporter and empty vector control ( n = 7 biological replicates). Bar: mean ± SE. *** P < 0.001 (Student’s two-tailed t -test). Source data underlying Fig. 2b–l are provided as a Source Data file. Full size image Y1H also showed that ATML1 and PDF2 proteins interact with the full-length promoter of MIR171B (Fig. 3a, b , Supplementary Fig. 1b ). We next found five putative binding sites of ATML1/PDF2 on the promoter sequence of the MIR171B gene, from either forward or reverse directions (Fig. 3a ), which all share at least six conserved base pairs of T (A/T)AATG with the previously identified L1 box [22] , [29] . We tested the binding of ATML1/PDF2 with each DNA fragment (from F1 to F5) that contains a putative binding site (Fig. 3a, c, d ), and we found that two fragments (F3 and F4) interact with ATML1 and PDF2 in Y1H (Fig. 3c, d ). We further confirmed the interaction between these two fragments and the recombinant GST ATML1 30–134 protein using EMSA, with both the GST and unlabeled competitor probes as the controls (Fig. 3e–h ). All the results consistently demonstrated that F3 and F4 with the core T (A/T)AATG sequence can interact with ATML1 but other fragments containing similar sequences cannot, suggesting that the flanking sequences of the T (A/T)AATG motif also contribute to the interaction between ATML1 and the DNA. In the dual-luciferase transactivation assay, we found that ATML1 can activate the pMIR171B::LUC reporter (Fig. 3i ), and the fold change of activation over the empty vector control (Fig. 3i ) is comparable to that in the assay with a pMIR171B::LUC::3 ′ MIR171B reporter (Supplementary Fig. 3 ). These results suggest that the 3′ regulatory region of MIR171B gene is dispensable for the activation of MIR171B by ATML1, although an additional L1 box from this region also interacts with both ATML1 and PDF2 (Supplementary Fig. 4 ). Taken together, our results demonstrated that ATML1 activates MIR171A and MIR171B through directly binding to their promoters. Fig. 3: ATML1 and PDF2 directly activate MIR171B . a Schematic structure of the MIR171B promoter. The expanded diagram shows the sequences of putative L1 boxes on the promoter. Probes indicate the DNA fragments used in the EMSA and Y1H. +1 indicates the transcription start site. b The full-length promoter of MIR171B interacts with ATML1 and PDF2 proteins in Y1H. Y axis: the relative activity of the pMIR171B::lacZ reporter. All the numbers are normalized to the average value of the empty vector control. Bars: mean ± SE ( n = 3 biological replicates). *** P < 0.001 (Student’s two-tailed t -test). c , d The MIR171B-F3 and MIR171B-F4 fragments from the MIR171B promoter interact with ATML1 ( c ) and PDF2 ( d ) proteins in Y1H. Y axis: the relative activity of each lacZ reporter when the empty vector control, ATML1 ( c ) or PDF2 (d) is present. All the numbers are normalized to the average value of the empty vector control. Bars: mean ± SE ( n = 5 biological replicates). *** P < 0.001 (Student’s two-tailed t -test). e – h EMSA shows that GST ATML1 [30] –134] but not GST binds to Cy5-labeled MIR171B-F3 probe ( e ) and MIR171B-F4 probe ( g ). The GST ATML1 [30] –134] –induced mobility shift of the Cy5-labeled MIR171B-F3 probe ( f ), and the Cy5-labeled MIR171B-F4 probe ( h ) can be chased away when excess amount of the unlabeled DNA probe (chase) is present. Arrows indicate free DNA probes and DNA-protein complexes. i Dual-luciferase assays show that ATML1 activates the transcription of MIR171B . Left panel: structure of the reporter construct. Right panel: LUC/REN, ratio of LUC to REN activity. The LUC/REN in the cells co-transformed with the reporter pMIR171B::LUC and the ATML1 effector ( n = 6 biological replicates) is significantly higher than that in the cells co-transformed with the same reporter and empty vector control ( n = 6 biological replicates). Bar: mean ± SE. *** P < 0.001 (Student’s two-tailed t -test). Source data underlying Fig. 3b–i are provided as a Source Data file. Full size image Besides MIR171A and MIR171B , ATML1 also binds to the promoters of MIR171C (Fig. 4a–c ) and MIR170 in the Y1H assays (Fig. 4d–f ). We found that one fragment (F1) from the MIR171C promoter (Fig. 4a ) and one fragment (F2) from the MIR170 promoter (Fig. 4d ) contain the T(A/T)AATG(C/T) sequence. Both fragments showed strong interactions with ATML1 in Y1H (Fig. 4c, f ). These results may explain why the expression of the MIR171C and MIR170 reporters is also specific in the epidermis of SAMs, though their expression levels are low (Fig. 1c, d ). Fig. 4: ATML1 binds to the promoters of MIR171C and MIR170 . a Schematic structure of the MIR171C promoter. The expanded diagram shows the sequences of putative L1 boxes on the promoter. Probes indicate the DNA fragments used in the Y1H assay. +1 indicates the transcription start site. b The full-length promoter of MIR171C interacts with ATML1 protein in Y1H. Y-axis: the relative activity of the pMIR171C::lacZ . All the numbers are normalized to the average value of the empty vector control. Bars: mean ± SE ( n = 5 biological replicates). *** P < 0.001 (Student’s two-tailed t -test). c The MIR171C-F1 fragment from the MIR171C promote interacts with the ATML1 protein in Y1H. Y-axis: the relative activity of the pMIR171C-F1::lacZ , pMIR171C-F2::lacZ and pMIR171C-F3::lacZ reporters. All the numbers are normalized to the average value of the empty vector control. Bars: mean ± SE ( n = 5 biological replicates). *** P < 0.001 (Student’s two-tailed t -test). d Schematic structure of the MIR170 promoter. The expanded diagram shows the sequences of putative L1 boxes on the promoter. Probes indicate the DNA fragments used in the Y1H assay. +1 indicates the transcription start site. e The full-length promoter of MIR170 interacts with ATML1 protein in Y1H. Y axis: the relative activity of the pMIR170::lacZ reporter. All the numbers are normalized to the average value of the empty vector control. Bars: mean ± SE ( n = 5 biological replicates). *** P < 0.001 (Student’s two-tailed t -test). f The MIR170-F2 fragment from the MIR170 promoter interacts with the ATML1 protein in Y1H. Y-axis: the relative activity of each lacZ reporter. All the numbers are normalized to the average value of the empty vector control. Bars: mean ± SE ( n = 5 biological replicates). *** P < 0.001 (Student’s two-tailed t -test). Source data underlying Fig. 4b, c and Fig. 4e, f are provided as a Source Data file. Full size image L1-box and ATML1/PDF2 are essential for regulating MIR171 To investigate whether these putative L1 box elements in the MIR171A promoter are essential for the epidermis specific expression of miR171, we mutated two L1-boxes in the MIR171A promoter and generated a pMIR171A-mut reporter (Supplementary Fig. 5 ). In the Y1H assay, these mutations significantly reduced the interaction between the pMIR171A promoter DNA and the ATML1 (Fig. 5a ) or PDF2 protein (Fig. 5b ). Furthermore, the mutations greatly reduced the activation of the pMIR171A-mut::LUC reporter by ATML1 in the transient dual-luciferase assays (Fig. 5c ). To further examine the biological significance of these L1 box elements in the MIR171A promoter, we introduced the pMIR171A-mut::H2B-GFP reporter in Arabidopsis (Supplementary Fig. 5 ). Compared to the expression of the pMIR171A::H2B-GFP control (Fig. 5d–g ), the pMIR171A-mut::H2B-GFP reporters showed reduced expression (Fig. 5h–k , Supplementary Fig. 6 ). Specifically, the majority of the independent transgenic lines we obtained (26 out of 31, 83.9%) showed no expression of the pMIR171A-mut::H2B-GFP reporter in SAMs but only weak expression in the epidermis of sepal primordia (Fig. 5h–k , Supplementary Fig. 6 ). Thus, we conclude that the L1 boxes mediate the activation of MIR171A by ATML1 and PDF2 in the epidermis of the SAMs and FMs. Fig. 5: Epidermis specific cis-regulatory elements are required for the activation of miR171. a , b Mutations in the MIR171A promoter significantly reduced its interaction with ATML1 ( a ) or PDF2 ( b ) in Y1H. Upper panel: sketch of the reporter used in the study. AD with no fusion protein was included as the control. The lacZ reporter was under the control of either the MIR171A promoter ( pMIR171A::lacZ ) or the MIR171A promoter with two sites of TTAAATGC mutated ( pMIR171A-mut::lacZ ). Lower panel: mutations in pMIR171A significantly reduced the activation of the pMIR171A::lacZ by ATML1 ( a ) or PDF2 ( b ). Bar: mean ± SE ( a : n = 5 biological replicates for AD control and AD-ATML1, except that n = 4 biological replicates for AD-ATML1 on pMIR171A-mut::lacZ ; b : n = 5 biological replicates for AD control and AD-PDF2). ** P < 0.01, *** P < 0.001 (Student’s two-tailed t -test). c Dual-luciferase assay shows that the activation of MIR171A promoter activities by ATML1 is greatly compromised by the two mutations in the MIR171A promoter. The LUC/REN in cells co-transformed with the pMIR171A::LUC reporter and the ATML1 effector ( n = 7 biological replicates) is significantly higher than that in tobacco cells co-transformed with the pMIR171A-mut::LUC reporter and the same effector ( n = 8 biological replicates). *** P < 0.001 (Student’s two-tailed t -test). d – g Expression of pMIR171A::H2B-GFP in an Arabidopsis SAM, from the orthogonal view ( d ), in the transverse optical section in corpus ( e ), and from the 3D projection view ( f , g ). h – k Expression of pMIR171A-mut::H2B-GFP in the SAM, from the orthogonal view ( h ), transverse optical section view in corpus ( i ), and from the 3D projection view ( j , k ). The confocal settings for imaging GFP in d – k are identical, and the quantification of GFP is indicated by the identical color bar in g , k . d , e , h , i : merge of GFP (green) and PI counterstain (purple); f , j : GFP (green); g , k : GFP quantified from f , j (quantification indicated by color). Scale bar: 20 µm; color bar in g , k : fire quantification of the signal intensity. Source data underlying Fig. 5a–c are provided as a Source Data file. Full size image To investigate whether ATML1 and PDF2 are required for the epidermis specific expression of the MIR171A and MIR171B , we introduced the pMIR171A::H2B-GFP reporter or the pMIR171B::H2B-GFP reporter into the atml1-1 pdf2-1 double mutant [23] through genetic crosses. Compared to the expression of pMIR171A::H2B-GFP and pMIR171B::H2B-GFP in wild type plants (Fig. 6a–e, k–o ), the expression levels of these two reporters were greatly reduced in atml1-1 pdf2-1 double mutant seedlings (Fig. 6f–j, p–t ). These results demonstrated that ATML1 and PDF2 are essential for the expression of MIR171A and MIR171B . Fig. 6: Epidermal specification pathway is required for the expression of MIR171 genes. a – e The wild type seedling (Col) expressing the pMIR171A::H2B-GFP reporter. f – j The atml1 pdf2 double mutant seedling expressing the pMIR171A::H2B-GFP reporter. k – o The wild type seedling (Col) expressing the pMIR171B::H2B-GFP reporter. p – t The atml1 pdf2 double mutant expressing the pMIR171B::H2B-GFP reporter. Panels (from left to right): seedlings used for the confocal imaging; DIC from one optical section; GFP (green) in 3D projection view, quantified GFP (quantification indicated by color) in 3D projection view; merge of GFP (green) and chlorophyll (red) in 3D projection view. Scale bars: 1 mm ( a , f , k , p ) and 100 µm ( b – e , g – j , l – o , and q – t ); color bar ( d , i , n , s ): fire quantification of the signal intensity. Full size image 3D computational model for the L1-miR171-HAM signal cascade Based on our results that ATML1/PDF2—the L1 specific transcription factors—directly activate miR171 transcription (Figs. 1 – 6 ) and the previous findings that miR171 directly silences HAM [11] , [12] , we hypothesized that there exists a L1-miR171-HAM signaling cascade, in which the epidermal ATML1/PDF2 determine the apical-basal concentration gradient of HAM in the SAM through the regulation of MIR171A/B . To test this hypothesis, we developed a computational model, which derives from our previously reported SAM model [9] , to help understand this signaling cascade in different cell layers in the three dimensional (3D) SAM. Different from the previous model, in which we used HAM concentration gradient as a key functional input [9] , we now used the epidermal specification factors, ATML1 and PDF2, as the key input. As an output, we simulated the concentration gradient of HAM in the SAM, as well as the MIR171 promoter activity and the patterns of miR171 (Supplementary Fig. 7 ). For simplicity of computational model, we first defined the functional ATML1 and its homolog PDF2 proteins as the input (ML1p), which are well-known to be L1-layer specific [20] , [21] . In the SAM of the wild-type plant, we set the concentration of ML1p 1 a.u. in cells of the L1 layer, and 0 a.u. in cells of the other layers. To model the dynamics of miR171, we set three conditions. First, the production of miR171 RNA is activated by the L1 layer specific ATML1 protein. As a result, miR171 is not produced in cells at the L2 and corpus layers in a wild type SAM. This condition is consistent with our experimental results described above (Fig. 1a–d ). Second, we set a constant degradation rate for miR171. Third, we set a low rescaled (by cell size) diffusion constant for the movement of miR171 from epidermis to deep layers. This condition is consistent with results from our RNA in situ hybridization experiments, which showed that the level of the endogenous miR171 is high in L1 and low in L2 and upper corpus layers (Supplementary Figs. 8 and 9 ). For the dynamics of HAM mRNA, we also set three conditions. First, the transcription of HAM mRNA is constitutively active in all layers of SAM. This is based on our finding that the transcriptional reporter of pHAM2::H2B-GFP lacking the miR171 binding site is highly expressed in all cell layers of the SAM (Fig. 1f ). Second, we set a constant rate for the miR171 independent HAM mRNA degradation. Third, miR171 activates the degradation of HAM mRNA, which is well supported by previous reports on the function of miR171 [11] , [12] , [13] . For the dynamics of HAM protein, we defined that the synthesis rate of HAM protein depends on the level of HAM mRNA, and the HAM protein is degraded at a constant degradation rate. In addition to miR171, HAM mRNA and HAM protein, the three key components, we also included an H2B-GFP transcriptional reporter to reflect the activity of the MIR171 promoter. Similar to miR171, the transcription of the H2B-GFP mRNA is activated by ATML1 protein, and the H2B-GFP mRNA is degraded at a constant rate. Further, the synthesis rate of the H2B-GFP reporter protein depends on the level of its mRNA, and it is degraded at a constant rate. Unlike miR171, which moves into deeper layers of the SAM, the H2B-GFP reporter cannot move between cells. Based on the model conditions mentioned above, we established five dynamic equations for miR171, HAM mRNA, HAM protein, H2B-GFP mRNA, and H2B-GFP protein, respectively (see details in Methods). In this model, the miR171 and HAM mRNA are essential for the apical-basal pattern of HAM gene expression. 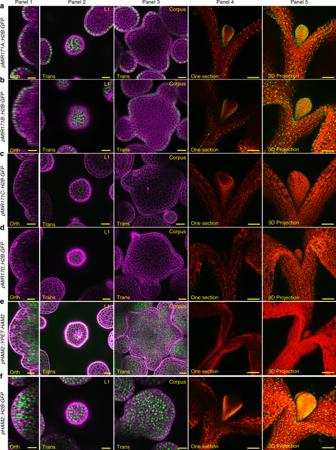Fig. 1: Epidermis expressedMIR170/171genes define the apical-basal gradient of HAM inArabidopsisSAMs. aThepMIR171A::H2B-GFPreporter is highly expressed at the epidermis in the SAM (panels 1–3) and in the young leaves (panels 4–5).bThepMIR171B::H2B-GFPreporter is highly expressed at the epidermis in the SAM (panels 1–3) and in the young leaves (panels 4–5).cThepMIR171C::H2B-GFPreporter is weakly expressed at the epidermis in the SAM (panels 1–3) and undetectable in the young leaves (panels 4–5).dThepMIR170::H2B-GFPreporter is weakly expressed at the epidermis in the SAM (panels 1–3) and in the young leaves (panels 4–5).eThepHAM2::YPET-HAM2reporter that is sensitive to the miR170/171 is expressed with a concentration gradient in the SAM, with high expression at inner cell layers and no expression in epidermis (panels 1–3). ThepHAM2::YPET-HAM2reporter is not expressed at the epidermis of the young leaves (panels 4–5).fThepHAM2::H2B-GFPreporter that is not sensitive to miR170/171 is highly expressed in all the cell layers (including the epidermal layer) in the SAM (panels 1–3), and thepHAM2::H2B-GFPreporter is highly expressed at the epidermis of the young leaves (panels 4–5). Panels (from left to right): 1, orthogonal view of a SAM; 2, transverse section view of L1 in the SAM; 3, transverse section view of corpus in the SAM; 4, section view of a seedling; 5, 3D projection view of the seedling. Channels: GFP/YFP (green), propidium iodide (PI) counterstain (purple), and Chlorophyll (red). Scale bar: (panels 1–3) 20 µm; (panels 4–5) 100 µm. Next, we set out to test whether the model can simulate the pattern of HAM mRNA in a wild-type SAM using one set of parameters (Supplementary Table 1 ), and we found that our model reproduced the typical apical (low)-basal (high) gradient of the HAM mRNA (Fig. 7m ). Fig. 7: The 3D computational model simulates the L1-miR171-HAM regulatory circuit in SAMs. a , b Input of the ATML1 level (L1 input) for the computational simulation in ( c , m ) and ( d , n ). Color indicates the level of ATML1 input, with the gradient from red (maximum, 1.1 a.u.) to blue (none). c , d Simulated promoter activity of MIR171 in the SAMs from the wild type control ( c ) and the plant with ectopic activation of ATML1 ( d ). Color indicates the simulated MIR171 reporter activity, with the gradient from red (maximum, 1.1 a.u.) to blue (none). e – h Confocal live imaging of the pMIR171B::H2B-GFP reporter in the SAMs of 35S::ATML1-GR plants, with the mock control ( e , f ) and the Dex treatment ( g , h ). Using identical imaging settings, the same SAM was imaged at 0 h and 24 h after the indicated treatment. Colors indicate quantified GFP intensities, and color bars represent fire quantification of signal intensity. Panels: (top) orthogonal view; (bottom) transverse optical section view from corpus. i – l Quantification of the gene expression for GFP ( i ), MIR171A ( j ), MIR171B ( k ), and HAM1 ( l ) in two independent 35S::ATML1-GR; pMIR171B::H2B-GFP transgenic lines (#5 and #9) 24 h after the mock or Dex treatment. Bars: mean ± SE. ** P < 0.01, *** P < 0.001 (Student’s two-tailed t -test). n = 3 biological replicates. m , n Simulated HAM1 mRNA expression patterns in SAMs from the wild type control ( m ) and the plant with ectopic activation of ATML1( n ). Color indicates the simulated HAM1 mRNA levels, with the gradient from red (at or above 2 a.u.) to blue (none). o , p RNA in situ hybridizations for HAM1 mRNA in the SAMs of 35S::ATML1-GR ; pMIR171B::H2B-GFP plants 5 days after the mock ( o ) or Dex ( p ) treatment. One set of representative results are shown, and similar results from three independent biological replicates were obtained for each treatment. Scale bar: 50 µm ( o – p ). The template of a whole SAM was used for all the simulations, and only a half of the SAM is displayed for visualization of cells in inner layers. Source data underlying Fig. 7i–l are provided as a Source Data file. 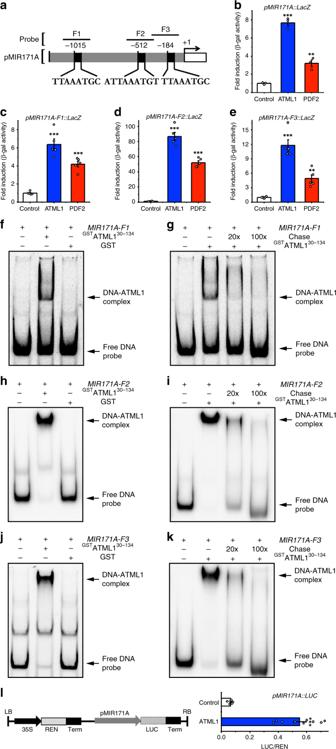Fig. 2: ATML1 and PDF2 directly activateMIR171A. aSchematic structure of theMIR171Apromoter. The expanded diagram shows the sequences of putative L1 boxes on the promoter. Probes indicate the DNA fragments used in the EMSA and the yeast one hybrid (Y1H) assay, and +1 indicates the transcription start site.bThe full-length promoter ofMIR171Ainteracts with ATML1 and PDF2 proteins in Y1H assays. Y-axis: the relative activity of thepMIR171A:: lacZreporter. All the numbers are normalized to the average value of the empty vector control. Bars: mean ± standard error (SE) (n= 3 biological replicates). **P< 0.01, ***P< 0.001 (Student’s two-tailedt-test).c–eDifferent DNA fragments from theMIR171Apromoter interact with ATML1 and PDF2 proteins in Y1H. Y-axis: the relative activity of thepMIR171A-F1::lacZ(c),pMIR171A-F2::lacZ(d) andpMIR171A-F3:: lacZ(e) reporters. All the numbers are normalized to the average value of the empty vector control. Bars: mean ± SE (n= 5 biological replicates). **P< 0.01, ***P< 0.001 (Student’s two-tailedt-test).f–kElectrophoretic mobility shift assay (EMSA) shows thatGSTATML130–134but not GST binds to the Cy5-labeled probes includingMIR171A-F1(f),MIR171A-F2(h) andMIR171A-F3(j). TheGSTATML130–134–induced mobility shift of the Cy5-labeled DNA probe can be chased away when excess amount of the unlabeled DNA probe (chase) is present (g,i,k). Arrows indicate free DNA probes and DNA-protein complexes.lDual-luciferase assays show that ATML1 activates the transcription ofMIR171A. Left panel: structure of the reporter construct. Term, CaMV terminator; LB, transfer DNA (T-DNA) left border; RB, T-DNA right border. Right panel: LUC/REN, ratio of firefly luciferase (LUC) to Renilla luciferase (REN) activity. The LUC/REN in tobacco cells co-transformed with the reporterpMIR171A::LUCand the ATML1 effector (n= 9 biological replicates) is significantly higher than that in the cells co-transformed with the same reporter and empty vector control (n= 7 biological replicates). Bar: mean ± SE. ***P< 0.001 (Student’s two-tailedt-test). Source data underlying Fig.2b–lare provided as a Source Data file. Full size image Our model contains six key parameters that control the dynamics of miR171 and the HAM mRNA expression patterns (Supplementary Table 2 ). We then explored the working ranges of these six key parameters surrounding the defined parameter values (Supplementary Table 2 ). In total, we found 235 sets of different combinations of parameter values (Supplementary Data 1 ). Using each set of parameter values, we can simulate patterns of HAM mRNA that are qualitatively comparable to the observed pattern in a wild-type SAM (Supplementary Movies 7 – 12 ), demonstrating the system we established is robust. These 235 sets of parameter values were also used in the sensitivity analyses for the six key parameters (Supplementary Fig. 10 ). We found that the total amount of HAM mRNAs shows higher sensitivity to changes in three of the six parameters, including k hrp and k hrnh that directly control the production and degradation of HAM mRNA, respectively, and k mirn that directly determines the degradation of miR171 (Supplementary Fig. 10 ). In addition to the local parameter search described above (Supplementary Table 2 , Supplementary Data 1 ), we further carried out unbiased random search for more diverse parameters in a 100-fold range (See Methods). We randomly sampled 20,000 sets of six different parameters uniformly on the log-scale (Supplementary Data 2 ) and ran simulations using each of 20,000 random parameter sets in the 3D template. We found that 173 new sets of solutions (Supplementary Data 3 ), which are different from the initial set of parameters (Supplementary Table 1 ), all lead to HAM mRNA expression patterns qualitatively comparable to the experimental observation in a wild type SAM (Supplementary Movie 13 ). We performed the sensitivity analyses for the six parameters again with the 173 new sets of parameter values, and the results (Supplementary Fig. 11 ) show the same tendencies for the parameter sensitivities compared to the analyses mentioned above (Supplementary Fig. 10 ). Evaluating the L1-miR171-HAM cascade in silico and in vivo To further study the regulatory cascade in the SAM, we computationally predicted the patterns of miR171 and HAM gene expression when the ATML1 protein is ectopically activated in the SAM. We first defined one set of [ML1p] input in the model based on the experimental results from the ATML1 RNA in situ hybridization (Supplementary Fig. 12 ). When ATML1 is ectopically activated, we set the level of ML1p 1.1 a.u. in the epidermal layer and 0.4 a.u. in sub-epidermal and corpus layers (see Methods for details), and we kept the values of all parameters the same for the simulation (Supplementary Table 1 ). As an output, the model shows that MIR171 promoter activity is increased in all layers of SAM while HAM mRNA levels are dramatically decreased in the SAM (Fig. 7a–d, m, n ). We then explored more ML1p input patterns and we found that 75 different ML1p input patterns all lead to dramatic reduction of HAM mRNA levels in all layers of SAM (Supplementary Movies 14 and 15 ), which is insensitive to differences of [ML1p] between epidermis and deeper layers, suggesting a robust response in the model for the ectopic activation of ATML1. In parallel, we tested these computational predictions experimentally (Fig. 7e–h , Supplementary Figs. 12 – 15 ). Because ATML1 drives the epidermal specification pathway and it regulates different sets of downstream targets and developmental processes [22] , [23] , [25] , [26] , [27] , [28] , prolonged activation of ATML1 will likely result in perturbations in a wide range of developmental events. Therefore, we decided to apply a dexamethasone (Dex) inducible transient activation system ( ATML1-GR ) to examine the immediate effects of ATML1 activation on the expression of MIR171 and HAM . We first introduced the 35S::ATML1-GR expression cassette in the pMIR171B::H2B-GFP reporter line, and then we performed the time-lapse live imaging of the pMIR171B::H2B-GFP reporter in the SAMs with either the mock or Dex treatment over a 24-h period. In the mock, seen from both the orthogonal view and transverse cross section view, the expression of the pMIR171B::H2B-GFP reporter in the same living SAM was specific in L1 at both 0 h (Fig. 7e ) and 24 h after the treatment (Fig. 7f ). In contrast, 24 h after the treatment of Dex, the pMIR171B::H2B-GFP signal in the living SAM was greatly induced in cells below the L1 layer (Fig. 7g, h ). In addition, through RNA in situ hybridization, we also detected the strong induction of pMIR171B::H2B-GFP reporter in the SAM and in the young leaves after the Dex treatment of the pMIR171B::H2B-GFP; 35S::ATML1-GR plant (Supplementary Fig. 14 ). The induced expression pattern (Supplementary Figs. 13 and 14 ) is comparable to the expression of ATML1 in the same pMIR171B::H2B-GFP; 35S::ATML1-GR line (Supplementary Fig. 12 ). Interestingly, using the similar procedure, we found that the pMIR171A::H2B-GFP reporter was also induced upon Dex treatment of the 35S::ATML1-GR line, with strong activation in young leaves but only mild and uneven induction in the SAM (Supplementary Fig. 15 ), suggesting potential differences in the regulation of the MIR171A promoter and the pMIR171B promoter in distinct cell types. In parallel, we found the transcript levels of GFP , MIR171A , and MIR171B in the 35S::ATML1-GR;pMIR171B::H2B-GFP plants were significantly increased in response to the Dex treatment compared with the mock control (Fig. 7i, j, k ). Taken together, consistent with the model predictions (Fig. 7c, d , Supplementary Fig. 16 ), our experiments demonstrated the immediate activation of MIR171 production by transient activation of ATML1 in vivo (Fig. 7e–l , Supplementary Figs. 12 – 15 ), supporting the first step of the proposed L1-miR171-HAM signaling cascade. To examine the second step of the L1-miR171-HAM signaling cascade, we performed the RNA in situ hybridization of HAM1 in the SAMs of the 35S::ATML1-GR plants with either mock or the Dex treatment at the same time using the identical procedure. The expression of HAM1 mRNA in the mock-treated SAM was consistent with the previous observation [6] , [7] , [9] , with a concentration gradient from the epidermis to the deep cell layers. The expression of HAM1 mRNA in the Dex-treated SAM was greatly reduced and was almost undetectable in the meristem and young leaf primordia (Fig. 7o, p ). Consistently, the qPCR experiments showed that the expression levels of HAM1 and HAM2 were significantly decreased in the Dex-treated 35S::ATML1-GR plants compared with the mock control (Fig. 7l , Supplementary Fig. 17 ). These results are consistent with the model prediction (Fig. 7m, n ) (Supplementary Movies 14 and 15 ). Taken together, both the modeling and experimental results support our proposed regulatory pathway, which starts from ATML1, transfers to miR171, and arrives at HAM, suggesting the epidermis-derived signal cascade shapes the concentration gradient of HAM in the SAM. Patterns of ATML1 and MIR171 in de novo stem cell niches In our previous work, we found that the de novo initiation of new meristem from leaf axils [30] also requires the concentration gradient of HAM [9] . Thus, we wondered whether the L1-miR171-HAM signaling cascade is also active in de novo axillary stem cell niches. We first performed the RNA in situ hybridization of ATML1 in the AMs from early to late stages during axillary meristem initiation (Fig. 8a–d ). ATML1 expression is not detectable at S1 (Fig. 8a ). However, it starts to appear in the epidermis as early as when a group of cells forming a bulge in the leaf axils (Fig. 8b ), and the expression continues in the epidermis at the stages thereafter (Fig. 8c, d ). In parallel, to probe the promoter activity of pMIR171A and pMIR171B , we performed the RNA in situ hybridizations of the GFP in the developing AMs at different stages from either the pMIR171A::H2B-GFP plants or the pMIR171B::H2B-GFP plants. The expression patterns of MIR171 from early to late stages are largely comparable to that of ATML1 (Fig. 8e–l ). These results together with our previous work [9] suggest a sequential regulation of gene expression during new meristem initiation: ATML1 is firstly activated at the early stage when the meristem identity is specified. Then, the miR171 expression is turned on in the epidermis. Consequently, the apical-basal concentration gradient of HAM is defined [9] , which shapes the CLV3 expression pattern and promotes the initiation of new stem cell niches [9] . Fig. 8: Pattern formation of L1 and miR171 in de novo axillary stem cell niches. a – d RNA in situ hybridization of ATML1 mRNA in wild-type (L er ) plants, from early to late developmental stages during the de novo formation of the axillary meristem (AM). e – h RNA in situ hybridization of GFP mRNA in pMIR171A::H2B-GFP plants showing the promoter activity of MIR171A , from early to late stages of AM initiation. i – l RNA in situ hybridization of GFP mRNA in pMIR171B::H2B-GFP plants showing the promoter activity of MIR171B , from early to late stages of AM initiation. The results have been confirmed by three biological replicates. Scale bar: 50 µm. Full size image With a high cellular resolution, we have revealed the expression patterns of all four MIR171/170 genes in Arabidopsis SAMs, which shows that miR171 originates from the epidermis during shoot development (Fig. 1 ). MIR171A and MIR171B genes are highly expressed in epidermis of the SAM (Fig. 1a, b ), whereas MIR171C and MIR170 genes are also specifically expressed in epidermis of the SAM but at a much lower level (Fig. 1c, d ). These results suggest that these four genes are responsible for the miR171 activity in the SAM and SAM derived leaves and flower meristems, while MIR171A and MIR171B genes contribute more to the total miR171 level in the SAM. Further, we found that MIR171 genes are the direct targets of both ATML1 and PDF2 transcription factors (Figs. 2 , 3 , and 7 ). It has been well documented that ATML1 and PDF2 recognize L1 box, the consensus cis-regulatory element, to regulate downstream targets [22] , [29] . We found that on the promoters of MIR171 genes, the (A)TT(A/T)AATG(C/T) sequences mediate the ATML1 binding. DNA sequences containing at least six base pairs of the conserved TAAATG may also function as the ATML1 binding sites, depending on the flanking sequences of each core element. These results are consistent with the previous studies on the sequence specificity and variation of the L1 box [22] , [24] , [29] . When two of the TTAAATGC L1 boxes were mutated, the expression of MIR171A was undetectable or largely reduced in the epidermis of the SAM, suggesting these L1 boxes are essential for the direct activation of MIR171 by ATML1/PDF2. Interestingly, the mutated MIR171A reporter was weakly expressed in the epidermis of flower sepal primordia (Fig. 5 ), suggesting there exists other cis-regulatory elements and/or transcriptional regulators that can activate MIR171 expression in developing organs. Indeed, it has been reported that MIR171 expression is reduced in the ham mutants [13] , [31] , and the MIR171 expression is also regulated by light [32] . Therefore, it is noteworthy to identify other factors contributing to the regulation of MIR171 expression in the future. We found that the miR171 insensitive transcriptional reporter ( pHAM2::H2B-GFP ) was expressed in all layers of the SAM. However, the miR171 sensitive translational reporter ( pHAM2::YFP-HAM2 ) was not detectable in the L1 layer, largely reduced in the L2 layer, and moderately reduced in upper corpus (Fig. 1e, f ). These results suggest that miR171 moves across at least two cell layers within the SAM, leading to a complete repression of HAM in L1, strong repression in L2, and moderate repression in cells located at upper corpus. Therefore, miR171 in SAMs serves as a mobile signal, and it shapes the HAM patterns not only in epidermis but also in inner cell layers. The movement of miRNA through limited distance in SAMs is not surprising, and it has been reported previously [33] , [34] . For example, when expressed in tunica (L1 and L2) layers, the movement of an artificial miRNA is limited and it only moves down one cell layer [33] . As another example, miR394b that is transcribed in the L1 layer of the SAM can form a concentration gradient with the movement through one or two cell layers [34] . Our finding together with these reports support the idea that the movement of microRNA through limited number of cell layers in the SAMs is likely an important feature for microRNAs to function. It will be interesting to further investigate the regulatory mechanism underlying the movement of miR171 among different cell layers. With the aid of a computational model, we established and simulated the key linkage from the epidermal signal (ATML1) to the concentration gradient of HAM in 3D SAMs. The transient activation of ATML1 results in quick and strong induction of MIR171 and the subsequently reduced HAM expression in the shoot, which was illustrated by both model simulation and live cell imaging. In the de novo axillary meristem, results presented here together with our previous work suggest that L1-miR171-HAM regulatory cascade is also active during the development of new axillary meristems (Fig. 8 ). ATML1 is not universally expressed at the epidermis throughout the whole plant body [20] , [21] , nor it is turned on at the leaf axis until a group of cells have acquired meristematic identity and start to form bulge (Fig. 8a, b ). When ATML1 is expressed, MIR171 starts to express at the epidermis of initiating meristems and remains its expression afterwards. This finding provides additional evidence supporting that ATML1 activates miR171, and it suggests that such regulation plays a role in the establishment of the concentration gradient of HAM and likely the apical-basal polarity of CLV3 expression as well [9] . The L1-miR171-HAM signaling cascade we proposed and validated in this study is specific to the SAMs and SAM derived young above-ground tissues, and all four MIR171/170 genes are not expressed at the epidermal layer of the roots, from the root cap to the differentiation zones (Supplementary Fig. 18 ). In contrast, the reporters of MIR171B and MIR171C are expressed in the inner layer at the differentiation zone in the root (Supplementary Fig. 18 ) (Supplementary Movies 16 and 17 ). Thus, the function and regulation of the miR171 family during the root development is still an open question. In summary, our work here uncovers the L1-miR171-HAM signal cascade during the shoot development. In the SAMs, this signal cascade determines the concentration gradient of HAM proteins, which are not present in epidermis but are regulated by signals initiated from the epidermis. Future study linking the L1-miR171-HAM signal cascade to various developmental processes mediated by HAM, including the previously proposed WUS-HAM-CLV3 regulatory loop, will provide a comprehensive view of this regulatory circuit in defining the plant shoot architecture. Plant materials and growth conditions Arabidopsis thaliana plants were grown in SunGro horticulture propagation mix soil under short-day conditions (8 h light/16 h dark cycle) at 22 °C, or continuous light at 22 °C. The atml1-1/+ pdf2-1 double mutant was previously described [7] , [23] . For the genotyping of atml1-1 pdf2-1 , a primer specific for the T-DNA left border (LB 5′- CATTTTATAATAACGCTGCGGACATCTAC-3′) was used in tandem with ATML1 -specific primers (5′-CCGGCTTGTGATCTTTCCG-3′ and 5′- GGCTCCGTCGCAGGCCAGAGC-3′) or PDF2 -specific primers (5′-ATTGATAGGATCTCTGCTATTG-3′ and 5′-CACATCCATGAGAATCTCAACGA-3′). Plasmid constructions for transgenic plants H2B-GFP was described previously [35] . To generate pMIR171A::H2B-GFP , 457 bp MIR171A 3′ terminator were amplified from Col-0 genomic DNA with primers 5′-TACAggcgcgccTCAGTACTCTCTCGTCTCTATTTT-3′ and 5′-TACAggcgcgccTGATTGTGACATTTTACATTGCTTC-3′ (restriction enzyme sites are in lower case) and cloned at 3′ of the H2B-GFP fragment to generate H2B-GFP-MIR171A-3 ′ terminator . Then 1474 bp MIR171A promoter was amplified using the primers 5′-ACAAgcggccgcGATACTCCACTTTTAGGCTCCATCTT-3′ and 5′-ACAAgcggccgcAAAGGGACTCTCTCATGCTTAAAG-3′ and inserted at the NotI site in front of the H2B-GFP-MIR171A-3 ′ terminator to get pMIR171A::H2B-GFP-MIR171A-3 ′ terminator . pMIR171A::H2B-GFP-MIR171A-3 ′ terminator fragment was then cloned into the binary vector pMOA34. For the construction of pMIR171B::H2B-GFP , 1852 bp MIR171B promoter was amplified with 5′-ACAAgcggccgcATATAAAACATGCTATTGCTTCTT-3′ and 5′-ACAAgcggccgcTAAAACCACTCTTGTTCGACTATAATC-3′ and cloned in front of H2B-GFP; and 960 bp 3′ terminator of MIR171B was PCR amplified with 5′-TACAggcgcgccAAGATAGTTATTATAACCTTAAAG-3′ and 5′-TACAggcgcgccGAGTCCTTATTGTTGTGCCTTTTTA-3′ and cloned 3′ of the H2B-GFP, then the fused DNA fragment was cloned into pMOA34. For the construction of pMIR171C::H2B-GFP , 2157-bp MIR171C promoter was amplified with 5′-ACAAgcggccgcTAATTCAAACCGAATTAGACCAAAA-3′ and 5′-ACAAgcggccgcTCGACTCTTCAGTTGCTTATTACACCA-3′ and cloned in front of H2B-GFP; and 1161 bp 3′ terminator of MIR171C was PCR amplified with 5′-TACAggcgcgccAATAGTTTAAAGATTCTATGTTAGTTG-3′ and 5′-TACAggcgcgccTGTAATTAAGATCTGCGACCACTTC-3′ and cloned at 3′ of the H2B-GFP fragment, then the fused DNA fragment was introduced into pMOA34. For the construction of pMIR170::H2B-GFP , 1251 bp MIR170 promoter was amplified with 5′-ACAAgcggccgcTCCTAACCTGTTCCTTTTGA-3′ and 5′-ACAAgcggccgcGAAACATAGTGTATCTGTTTTGTAA-3′ cloned in the front of H2B-GFP; and 582 bp 3′ terminator of MIR170 was PCR amplified with 5′-TACAggcgcgccTCGCTTCTCTCGTATTTTGAA-3′ and 5′-TACAggcgcgccGCTCCACCACAAAGCTCTTC-3′ and cloned at 3′ of the H2B-GFP fragment, then the fused DNA fragment was introduced into pMOA34. The promoter and 3′ terminator of pHAM2::H2B-GFP were the same as that in the pHAM2::YPET-HAM2 construct described before [9] . The above described constructs were transformed into L er through floral dip [36] , except the pHAM2::YPET-HAM2 construct, which was transformed into ham123 triple mutants. The pMIR171A::H2B-GFP and pMIR171B::H2B-GFP constructs were also transformed into Col. The expression patterns of each construct were confirmed in multiple lines. To construct of pMIR171A-mut::H2B-GFP , two L1 boxes in the MIR171A promoter were mutated from TTAAATGC to CCCGGTGC (Supplementary Fig. 5 ) using two round of overlapping PCR [37] . For the first round of overlapping PCR, the primers 5′- AGTAGTAGCTTAATATCAATGTCGCACCGGGGGAACATTATAAGCTACTAATATGAAA-3′, and 5′-TTTCATATTAGTAGCTTATAATGTTCCCCCGGTGCGACATTGATATTAAGCTACTACT-3′ were used to mutate the L1 box located at distal end (F1) of MIR171A promoter. For the second round of overlapping PCR, the primers 5′-AGGAAATGGAAGGTATGGAGCACCGGGACCTCATCTACTACCAAAGCACAAA-3′ and 5′-TTTGTGCTTTGGTAGTAGATGAGGTCCCGGTGCTCCATACCTTCCATTTCCT-3′ were used to mutate the L1 box located at proximal end (F3) of MIR171A promoter. The mutations have been confirmed through the sequencing. pMOA34 pMIR171A-mut:H2B-GFP was transformed to L er through flower dipping [36] . To generate 35 S::ATML1-GR , ATML1 cDNA was amplified using the primers 5′- CATAgagctcATGTATCATCCAAACATGTTCGA-3′ and 5′-AGTTgagctcTGGTGGTGCTGCTGCTGCTGCTGCGGCTCCGTCGCAGGCCAGAGCGG-3′ (restriction enzyme sites are indicated in lower case and underlined is the linker) into the SacI site of pGreen0029 35S::GR. pGreen0029 35S::ATML1-GR was transformed into the pMIR171A::H2B-GFP line 14 and the pMIR171B::H2B-GFP line 3 in L er background. Confocal live imaging All of the florescence reporters were imaged using a Zeiss LSM 880 upright confocal microscope. The live-imaging experiments were performed as previously described [7] , [38] , [39] . The shoot apices including SAMs were imaged with the water dipping lens (Zeiss). To image GFP and PI simultaneously in the SAMs and roots or to image GFP and chlorophyll simultaneously in the young seedlings, the GFP, chlorophyll or PI was excited using a 488-nm laser line. To image YPET and PI simultaneously in the SAMs or YPET and chlorophyll simultaneously in the young seedlings, YPET, chlorophyll or PI was excited by a 514-nm laser line. To image pMIR171A::H2B-GFP , pMIR171B::H2B-GFP , pMIR171C::H2B-GFP , pMIR170::H2B-GFP , pHAM2::H2B-GFP and pHAM2::YPET-HAM2 reporters, the shoots from 9-day-old seedlings grown in short days and the inflorescence shoot apices from the bolted plants were used (Fig. 1 ). To examine the expression of MIR171A and MIR171B in the atml1-1 pdf2- 1 double mutant, the pMIR171A::H2B-GFP reporter (line 11) and the pMIR171B::H2B-GFP reporter (line 5) in Col background were crossed into atml1-1/+ pdf2-1 mutants [23] . Within the F2 population, the atml1-1/+ pdf2-1 lines were identified and maintained through the PCR based genotyping and the expression of the reporter was confirmed through confocal imaging. Multiple F3 generation plants of pMIR171A::H2B-GFP in atml1-1/+ pdf2-1 and pMIR171B::H2B-GFP in atml1-1/+ pdf2-1 background were first grown on hygromycin plates to identify the lines containing the homozygous reporter. Then the identified lines with the homozygous reporter were grown on half MS media for 5 days in short day. The seedlings with the previously described atml1-1 pdf2-1 phenotype (no cotyledons) [23] were identified as the double homozygous mutants and imaged together with the homozygous reporter in wild type using confocal microscope, and several individual seedlings of these atml1-1 pdf2-1 double mutants have been confirmed through the genotyping PCR. To investigate the expression of MIR171B in response to the transient activation of ATML1 in Arabidopsis, the 35S::ATML1-GR; pMIR171B::H2B-GFP plants were grown in short days for 25 days and then moved to continuous light to induce flowering. The inflorescence shoot apices were dissected out and mounted in the GM media supplemented with B5 vitamins, and the SAMs were live-imaged at both 0 hour and 24 h after mock or the 10-µM Dex treatment. The live imaging results in this study have been confirmed using two independent 35S::ATML1-GR; pMIR171B::H2B-GFP lines (lines 5 and 9) with more than three biological replicates from each line. All the images were processed and quantified in Fiji. Protein expression and purification GST or GST ATML 30–134 proteins were expressed and purified following the same procedure as previously reported [7] , [40] . Briefly, an empty pGEX vector or a pGEX vector carrying the open reading frame of ATML 30–134 was transformed in Rosetta E. coli cells. Expression of the recombinant proteins were induced with 0.2 mM IPTG at 16 °C overnight. The expressed GST or GST ATML 30–134 proteins were extracted from the E. coli cells using Glutathione Sepharose resins (GE healthcare). Proteins eluted from the resins were further purified using size exclusion chromatography, and eluate fractions containing the protein of interest were combined and used for the study (Supplementary Fig. 2 ). Gel mobility shift assay (EMSA) Cy5-labeled DNA fragments were used as probes for EMSA. The labeled DNA probes were synthesized through regular PCR using oligos conjugated with Cy5 at the 5′ end (synthesized and purified by IDT). The DNAs were then purified (Qiagen) and stored in amber tubes at −20 °C before use. The MIR171A probe F1 (Fragment 1) (Fig. 2a, f, g ) was amplified from Col-0 genomic DNA using the primers 5′-ATGTGAATGAAGCCAAGAATCA-3′ and 5′-TTTCTTTTCAGGATTACTGTTTTCG-3′. The MIR171A probe F2 (Fragment 2) (Fig. 2a, h, i ) was amplified from Col-0 genomic DNA using the primers 5′-GGGTTCATAACTTGCTTGAGG−3′ and 5′-TTTCCTTCTTGAGGAGGTTCA-3′. The MIR171A probe F3 (Fragment 3) (Fig. 2a, j, k ) was amplified from Col-0 genomic DNA using the primers 5′-CCTCCTCAAGAAGGAAAGACAG-3′ and 5′-AGTGAGAATGTCTGTGGGGAGT-3′. The MIR171B probe F3 (Fragment 3) (Fig. 3a, e, f ) was amplified from Col-0 genomic DNA using the primers 5′-ATGTTGATTACCCATATACTTTGCT-3′ and 5′-TCCCACGAGCTTTCAATTTAGT-3′. The MIR171B probe F4 (Fragment 4) (Fig. 3a, g, h ) was amplified from Col-0 genomic DNA using the primers 5′-CCTGATAATTTGATATCATCGGTTG-3′ and 5′-ATGCGGCCAGTAGCAAAGT-3′. When assaying the gel mobility shift, 7.5 nM Cy5-labeled DNA probe in buffer containing 15 mM Tris (pH 7.5), 50 mM NaCl, 0.1 mM DTT, 5% glycerol, 0.1 mM MgCl 2 , and 50 ng/µl carrier DNA (Invitrogen) was first incubated with GST or GST ATML 30–134 protein at room temperature for 30 min. The mixture was subsequently fractionated on a 6% DNA Retardation Gel (ThermoFisher Scientific) in running buffer containing 0.5x TBE at 4 °C for 1 h with 100 V power supplied. Gels were scanned by a Typhoon FLA 9500 gel imaging scanner (GE Healthcare) to detect the Cy5-labeled DNA probe. To confirm the interaction between the DNA probe and the GST ATML 30–134 protein, a chase assay was performed by adding excess amount of unlabeled DNA with identical sequence to the fluorescent probe. The unlabeled DNA was added together with the labeled DNA probe before the addition of the GST ATML 30–134 protein. The subsequent steps were the same as described above. All the EMSA experiments in this study were repeated two times and they showed the same results. RNA in situ hybridization RNA in situ hybridization were performed as previously described [9] . Plant samples were fixed in 4% paraformaldehyde in phosphate-buffered saline (PBS) at 4 °C overnight. Then the samples were embedded in Paraplast X-Tra (McCormic Scientific) and sectioned with 8 µm thickness using a microtome (Thermo Scientific). Sections were transferred to microslides and dried overnight at 42 °C on a slide warmer. Sections were dewaxed and treated at 0.2 M HCl for 20 min, followed by 2 x SSC for 15 min at 70 °C. Then the sections were treated with Protease K (1 µg/ml) for 30 min, followed by 0.1 M thiethanolamine (pH 8.0) and 0.5% acetic anhydride for 10 min. Probes were mixed with the hybridization solution (50% formamide, 300 mM NaCl, 10 mM Tris-pH7.5, 1 mM EDTA, 1x Denhardts solution, 10% Dextron Sulfate, 70 mM DTT, 150 µg/ml tRNA). Samples were hybridized with the indicated probe in the hybridization solution at 53 °C overnight, and the sample slides were washed with 0.2 x SSC four times (30 min each wash) at 53 °C. Thereafter, slides were blocked with 1% Blocking Reagent (Roche) in PBS containing 0.3% Triton X-100 for 45 min, followed by incubation with 1% bovine serum albumin (BSA) in PBS containing 0.3% Triton X-100 for 45 min. Immuno-detection of the hybridized probe was performed by incubating slides with the 0.5% BSA/PBS/0.3% Triton X100 solution containing the anti-DIG antibody (1:1000 dilution) for 3 h. After that, the slides were washed with PBS and buffer containing 100 mM Tris pH 9.5, 100 mM NaCl, and 50 mM MgCl 2 . For signal visualization, slides were developed using Western blue stabilized substrate for alkaline phosphatase (Promega). The probe for GFP was cloned into pGEM-T easy (Promega) using the primers: 5′-CAAGGGCGAGGAGCTGTT-3′ and 5′-CTTGTACAGCTCGTCCATGC-3′. The probe for HAM1 was described previously [9] . The probe for ATML1 was cloned into pGEM-T easy (Promega) using the primers: 5′-ACTGGCGTAGCAGGGAACTA-3′ and 5′-GGCTCCGTCGCAGGCCAGAGC-3′. Probes were in vitro transcribed in the presence of DIG-UTP using the Sp6/T7 transcription kit (Roche). The synthesized probes were hydrolyzed in Carbonate hydrolysis buffer (60 mM Na 2 CO 3 and 40 mM NaHCO 3 ) at 60 °C. To investigate the expression patterns of GFP in the SAMs of the 35S::ATML1-GR; pMIR171A::H2B-GFP plant with mock or the Dex treatment, the 35S::ATML1-GR; pMIR171A::H2B-GFP plants were grown in short days for 24 days. Then they were sprayed with mock (no Dex) or with 10 µM Dex solution. At 24 h after mock or the Dex treatment, vegetative SAMs were collected for RNA in situ hybridization to GFP . This experiment was confirmed with three biological replicates. To investigate the expression patterns of GFP and HAM1 in the SAMs of the 35S::ATML1-GR; pMIR171B::H2B-GFP plant with mock or the Dex treatment, the 35S::ATML1-GR; pMIR171B::H2B-GFP plants (line 9) were grown in short days for 21 days. Then they were sprayed with mock (no Dex) or with 10 µM Dex solution every the other day. At 5 days after mock or the Dex treatment, vegetative SAMs were collected for RNA in situ hybridization to GFP and HAM1 . RNA in situ hybridization to GFP was confirmed with two biological replicates, and RNA in situ hybridization to HAM1 was confirmed with three biological replicates. To investigate the localization of miR171 in the wild type SAMs, the DIG labeled miRCURY Locked Nucleic Acid (LNA) miRNA detection probe (5′-CGTGATATTGGCACGGCTCA-3′) of miR171b (Qiagen) was used. The DIG labeled miRCURY LNA miRNA detection probe (5′-TCAAGGTCCGCTGTGAACAC-3′) of miR124 (Qiagen), which specifically recognizes murine miR124, was used as the negative control as previously suggested [41] , [42] . The RNA in situ hybridization was performed using our standard protocol of RNA in situ hybridization for mRNAs, except that the LNA probes for miR171 and for miR124 were prepared in 50% formamide and heated for 3 min at 85 °C following the same procedure (step 11) described in the published protocol [41] . Both LNA probes were used with the concentration of 100 nM and at 53 °C hybridization temperature. Inflorescences were collected from Ler wild type plants that were grown in short day for 28 days and then continuous light for 17 days (Supplementary Fig. 8 ). These experiments were repeated with four biological replicates for each probe at the same time with the identical procedure. To harvest vegetative SAMs, Ler wild type plants were grown in short days (Supplementary Fig. 9 ). These experiments were repeated with five independent biological replicates. To investigate the expression patterns of ATML1 in the SAMs of the L er wild type and the 35S::ATML1-GR; pMIR171B::H2B-GFP plant (line 9), the plants were grown in short days for 23 days. RNA in situ hybridization to ATML1 was performed using the identical procedure. This experiment was confirmed with three biological replicates for each genotype. To investigate the expression pattern of ATML1 during AM (axillary meristem) initiation, wild type L er plants were grown in short days for 28 days and then in continuous light for 1–2 days. All these experiments were repeated with three biological replicates. To investigate the expression pattern of pMIR171A::H2B-GFP and pMIR171B::H2B-GFP during AM (axillary meristem) initiation, pMIR171A::H2B-GFP line 14 and pMIR171B::H2B-GFP line 3 were grown in short days for 28 days and then in continuous light for 1–2 days. All these experiments were repeated with three biological replicates. Transactivation assay in tobacco To generate a pMIR171A::LUC reporter, the same MIR171A promoter described above was PCR amplified from Col-0 genomic DNA with the primers 5′-ACGGggtaccGATACTCCACTTTTAGGCTCCATCTT-3′ and 5′-ACGCgtcgacAAAGGGACTCTCTCATGCTTAAAG-3′ (restriction enzyme sites are in lower case) and cloned with KpnI and SalI into pGREEN800II-LUC [43] . To generate a pMIR171A-mut::LUC reporter, the MIR171A-mut promoter was PCR amplified with the primers 5′-ACGGggtaccGATACTCCACTTTTAGGCTCCATCTT-3′ and 5′-ACGCgtcgacAAAGGGACTCTCTCATGCTTAAAG-3′ and cloned with KpnI and SalI into pGREEN800II-LUC [43] . To generate a pMIR171B::LUC reporter, the MIR171B promoter was amplified with the primers 5′-ACGGggtaccATATAAAACATGCTATTGCTTCTT-3′ and 5′- ACGCgtcga C TAAAACCACTCTTGTTCGACTATAATC-3′ and cloned with KpnI and SalI into pGREEN800II-LUC. To generate a pMIR171B::LUC::MIR171B 3 ′ -terminator reporter, the MIR171B promoter was amplified with the primers 5′-ACGGggtaccATATAAAACATGCTATTGCTTCTT-3′ and 5′-ACAAgcggccgcTAAAACCACTCTTGTTCGACTATAATC-3′ and cloned with KpnI and NotI into pGREEN800II-LUC to generate pMIR171B::LUC . Then the MIR171B 3′ terminator was PCR amplified from Col-0 genomic DNA with primers 5′-CTAGtctagaAAGATAGTTATTATAACCTTAAAG-3′ and 5′- CTAGtctagaGAGTCCTTATTGTTGTGCCTTTTTA-3′ and cloned with XbaI into pMIR171B::LUC to get pMIR171B::LUC::MIR171B 3 ′ -terminator . The effector ATML1 (35S::ATML1-GFP) was generated by introducing ATML1 cDNA into pMDC83. These dual-luciferase reporter constructs and indicated effectors (empty vector or ATML1) were introduced into N. benthamiana leaves through Agrobacterium infiltration. The activities of firefly luciferase (LUC) and Renilla luciferase (REN) were quantified 2 days after infiltration with a Dual Luciferase Assay kit (Promega), and luminescence was recorded using a 96-well Iuminometer (Tecan). The LUC activity was normalized to the REN activity (LUC/REN). The means and standard errors of LUC/REN were calculated from indicated numbers of biological replicates that are described in the figure legends. Each set of experiment has been independently repeated at least two times. Yeast one hybrid To generate the reporters of pMIR171A::lacZ , pMIR171A-mut::lacZ , and pMIR171B::lacZ , the promoter of MIR171A , the mutated promoter of MIR171A (named as MIR171A-mut ) and the promoter of MIR171B was subcloned, respectively with KpnI and SalI into pLacZi (Clontech). To generate the pMIR171A-F1::lacZ reporter, the fragment 1 (F1) of the MIR171A promoter was amplified with the primers 5′- ACGGggtaccATGTGAATGAAGCCAAGAATCA-3′ and 5′- ACGCgtcgacTTTCTTTTCAGGATTACTGTTTTCG-3′ and cloned with KpnI and SalI into pLacZi. To generate the pMIR171A-F2::lacZ reporter, the fragment 2 (F2) of the MIR171A promoter was amplified with the primers 5′-ACGGggtaccGGGTTCATAACTTGCTTGAGG-3′ and 5′-ACGCgtcgacTTTCCTTCTTGAGGAGGTTCA-3′ and cloned with KpnI and SalI into pLacZi. To generate the pMIR171A-F3::lacZ reporter, the fragment 3 (F3) of the MIR171A promoter was amplified with the primers 5′- ACGGggtaccCCTCCTCAAGAAGGAAAGACAG-3′ and 5′- ACGCgtcgacAGTGAGAATGTCTGTGGGGAGT−3′ and cloned with KpnI and SalI into pLacZi. To generate the pMIR171B-F1::lacZ reporter, the fragment 1 (F1) of the MIR171B promoter was amplified with the primers 5′-ACGGggtaccATATAAAACATGCTATTGCTTCTT-3′ and 5′-ACGCgtcgacCAAGTACCCAAAAACACTGAAAAA-3′ and cloned with KpnI and SalI into pLacZi. To generate the pMIR171B-F2::lacZ reporter, the fragment 2 (F2) of the MIR171B promoter was amplified with the primers 5′-ACGGggtaccTGCAAAGTCAATTATTTCTTTAAGC-3′ and 5′-ACGCgtcgacTCGGCCGCTAGCAAAGTAT-3′ and cloned with KpnI and SalI into pLacZi. To generate the pMIR171B-F3::lacZ reporter, the fragment 3 (F3) of the MIR171B promoter was amplified with the primers 5′-ACGGggtaccATGTTGATTACCCATATACTTTGCT-3′ and 5′-ACGCgtcgacTCCCACGAGCTTTCAATTTAGT-3′ and cloned with KpnI and SalI into pLacZi. To generate the pMIR171B-F4::lacZ reporter, the fragment 4 (F4) of the MIR171B promoter was amplified with the primers 5′-ACGGggtaccCCTGATAATTTGATATCATCGGTTG-3′ and 5′-ACGCgtcgacATGCGGCCAGTAGCAAAGT-3′ and cloned with KpnI and SalI into pLacZi. To generate the pMIR171B-F5::lacZ reporter, the fragment 5 (F5) of the MIR171B promoter was amplified with the primers 5′-ACGGggtaccCTTGCTTGCCTCTCTTCTTCA-3′ and 5′-ACGCgtcgacCCACTTAGCTCCAGAAAACCA-3′ and cloned with KpnI and SalI into pLacZi. To generate the pMIR171B-F6::lacZ reporter, the fragment 6 (F6) from the 3′ region of the MIR171B gene was amplified with the primers 5′-ACGGggtaccTTTCATCAAGTCGGTCCACA-3′ and 5′-ACGCgtcgacATCGATCGCATCTTTGGATT-3′ and cloned with KpnI and SalI into pLacZi. To generate the pMIR171C::lacZ reporter, the promoter of MIR171C was amplified with the primers 5′-ACGGggtaccTAATTCAAACCGAATTAGACCAAAA-3′ and 5′-ACGCgtcgacTCGACTCTTCAGTTGCTTATTACACCA-3′ and cloned with KpnI and SalI into pLacZi. To generate the pMIR171C-F1::lacZ reporter, the fragment 1 (F1) of the MIR171C promoter was amplified with the primers 5′-ACGGggtaccCATGCACTATTCATAGACCCATGT-3′ and 5′-ACGCgtcgacTCATGCATAAGCTTGCTTGG-3′ and cloned with KpnI and SalI into pLacZi. To generate the pMIR171C-F2::lacZ reporter, the fragment 2 (F2) of the MIR171C promoter was amplified with the primers 5′- ACGGggtaccTTTCTTCATCACCCTCTTCG-3′ and 5′- ACGCgtcgacTCGACTCTTCAGTTGCTTATTACACCA-3′ and cloned with KpnI and SalI into pLacZi. To generate the pMIR171C-F3::lacZ reporter, the fragment 3 (F3) from the 3′ region of the MIR171C gene was amplified with the primers 5′- ACGGggtaccCCATGAACTAACCAGACGATCA-3′ and 5′- ACGCgtcgacTGTAATTAAGATCTGCGACCACTTC-3′ and cloned with KpnI and SalI into pLacZi. To generate the pMIR170::lacZ reporter, the promoter of MIR170 was amplified with the primers 5′-GCCCaagcttTCCTAACCTGTTCCTTTTGA-3′ and 5′-ACGCgtcgacGAAACATAGTGTATCTGTTTTGTAA-3′ and cloned with HindIII and SalI into pLacZi. To generate the pMIR170-F1::lacZ reporter, the fragment 1 (F1) of MIR170 promoter was amplified with the primers 5′-GCCCaagcttGGTGGATTTCAAGGGTATGG-3′ and 5′-ACGCgtcgacAACCGTCCCTCTTTCGTTTT-3′ and cloned with HindIII and SalI into pLacZi. 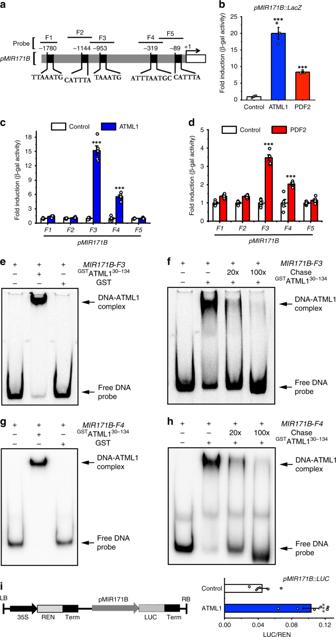Fig. 3: ATML1 and PDF2 directly activateMIR171B. aSchematic structure of theMIR171Bpromoter. The expanded diagram shows the sequences of putative L1 boxes on the promoter. Probes indicate the DNA fragments used in the EMSA and Y1H. +1 indicates the transcription start site.bThe full-length promoter ofMIR171Binteracts with ATML1 and PDF2 proteins in Y1H. Y axis: the relative activity of thepMIR171B::lacZreporter. All the numbers are normalized to the average value of the empty vector control. Bars: mean ± SE (n= 3 biological replicates). ***P< 0.001 (Student’s two-tailedt-test).c,dTheMIR171B-F3andMIR171B-F4fragments from theMIR171Bpromoter interact with ATML1 (c) and PDF2 (d) proteins in Y1H. Y axis: the relative activity of eachlacZreporter when the empty vector control, ATML1 (c) or PDF2 (d) is present. All the numbers are normalized to the average value of the empty vector control. Bars: mean ± SE (n= 5 biological replicates). ***P< 0.001 (Student’s two-tailedt-test).e–hEMSA shows thatGSTATML130–134]but notGSTbinds to Cy5-labeledMIR171B-F3probe (e) andMIR171B-F4probe (g). TheGSTATML130–134]–induced mobility shift of the Cy5-labeledMIR171B-F3probe (f), and the Cy5-labeledMIR171B-F4probe (h) can be chased away when excess amount of the unlabeled DNA probe (chase) is present. Arrows indicate free DNA probes and DNA-protein complexes.iDual-luciferase assays show that ATML1 activates the transcription ofMIR171B. Left panel: structure of the reporter construct. Right panel: LUC/REN, ratio of LUC to REN activity. The LUC/REN in the cells co-transformed with the reporterpMIR171B::LUCand the ATML1 effector (n= 6 biological replicates) is significantly higher than that in the cells co-transformed with the same reporter and empty vector control (n= 6 biological replicates). Bar: mean ± SE. ***P< 0.001 (Student’s two-tailedt-test). Source data underlying Fig.3b–iare provided as a Source Data file. To generate the pMIR170-F2::lacZ reporter, the fragment 2 (F2) of the MIR170 promoter was amplified with the primers 5′-GCCCaagcttACGAAAGAGGGACGGTTACA-3′ and 5′-ACGCgtcgacACTGTAAGGAGATTAAGAAGAAGAAGG-3′ and cloned with HindIII and SalI into pLacZi. To generate the pMIR170-F3::lacZ reporter, the fragment 3 (F3) from the 3′ region of the MIR170 gene was amplified with the primers 5′- GCCCaagcttATCGGATGCTCCTTTCTCCT-3′ and 5′- ACGCgtcgacCCAAGAATGGCCTTCCTACA-3′ and cloned with HindIII and SalI into pLacZi. To generate the reporter strains, each pLacZi construct described above was transformed and integrated into the yeast YM4271 (Clontech). ATML1 and PDF2 cDNAs were cloned into pENTR-D-TOPO gateway entry vector (invitrogen) and then cloned into pDEST22 through LR reaction. These effector constructs were then transformed into each yeast reporter strain. The β-galactosidase (β-gal) activity was quantified using ONPG as substrate and in 96-well plate reader (Tescan) as previously described [44] . The fold of induction is calculated based on the β-gal activities for each transcription factor normalized to that from the empty vector controls. The means and standard errors of relative β-gal activities were calculated from indicated numbers of biological replicates that are described in the figure legends. Regarding the fold of induction in all the quantitative assays in Y1H, the cutoff line was set as two and any value less than two was not considered as positive interaction. The x-gal lifting assay was performed as previous described [45] . Each set of experiment has been independently repeated two times. Computational modeling and simulation The current computational model is simulated on the same dome-shaped template (1216 overlapping spheres to mimic the SAM of Arabidopsis) [9] . The cell positions, cell sizes, and cell neighbors are defined in the 3D template [9] . Neighboring cells were identified by searching for the overlaps among spheres. Similar multiple spheres based 3D templates have been developed and used in previous modeling research on the transcriptional circuits and gene expression patterns involving WUS , CLV3 , HAM , and/or hormone cytokinin in the SAM [8] , [46] , [47] , [48] . Since this model focuses on the gene expression patterns in the SAM and there is no clear experimental evidence for fluxes of the gene products ( ATML1 , miR171 , and HAM ) into and/or out of Arabidopsis SAMs, the boundary condition for this current model is set to be no flux boundary [9] . Dynamics of three key native molecules, namely microRNA171 ([ miR171 ]), HAM mRNA ([ HAMr ]), and HAM protein ([ HAMp ]) are described using the system of differential Eqs. ( 1 )–( 3 ). To simulate the H2B-GFP reporter for MIR171 transcriptional activity, we added two more equations for simulation of the patterns of the pMIR171 reporter, which can be compared with and validated by our experimental data from confocal imaging of this reporter line. Since H2B-GFP only function as a reporter, there is no feedback regulation from the H2B-GFP reporter to the other components in the system described in Eqs. ( 1 )–( 3 ). The equations are applicable to each of the cells in the template, and the cell indices are omitted in the equations as shown. Relations among different agents are illustrated in the schematic diagram (Supplementary Fig. 7 ). d[miR171]/dt = k_mirp[ ML1p] - k_mirn[ miR171] + D_mir171Δ[ miR171]
 (1) 
    d[HAMr]/dt = k_hrp - k_hrnm[ HAMr][ miR171] - k_hrnh[ HAMr]
 (2) 
    d[HAMp]/dt = k_hpp[ HAMr] - k_hpn[ HAMp]
 (3) 
    d[GFPr]/dt = k_grp[ ML1p] - k_grn[ GFPr]
 (4) 
    d[GFPp]/dt = k_gpp[ GFPr] - k_gpn[ GFPp]
 (5) Equation ( 1 ) describes dynamics of miR171. k mirp is the parameter for miR171 production. [ML1p] is the concentration of functional ATML1 and its homolog PDF2 proteins. We assumed that miR171 production is activated by ATML1 and its homolog. This assumption is supported by four lines of evidence from our experimental results in this study: (1). ATML1 protein directly binds to the MIR171 promoters; (2). The MIR171 transcriptional reporter is induced by ATML1 in tobacco cells. ; (3). The expression of the MIR171 transcriptional reporter in epidermis is lost in atml1 pdf2 double mutant plants; (4). Mutations in the ATML1 binding sites in the MIR171A promoter result in the abolishment of activation of MIR171 transcriptional reporter both in the transient activation assays and in the SAM. k mirn is the parameter for miR171 degradation, and we assumed a constant rate for miR171 degradation throughout the SAM. In the third term of Eq. ( 1 ), we assumed that the epidermis produced miR171 RNA will move into deeper layers with a low diffusion constant, leading to a high to low gradient of miR171 RNA from the epidermal layer to deeper layers in the SAM. This assumption is supported by the results from the RNA in situ hybridization experiments to probe the miR171 localization in the SAM (Supplementary Figs. 8 and 9 ). \(D_{mir171}\) is the rescaled diffusion constant (rescaled by cell size) of miR171 among SAM cells. \(\Delta\) is the discrete Laplace operator, and the contribution of \(\Delta \left[ {miR171} \right]\) to the derivative for miR171 RNA in cell i is given by \(\mathop {\sum }\nolimits_n (\left[ {miR171} \right]_n \, - \, \left[ {miR171} \right]_i)\) , where the sum is over neighboring cells. The set of neighbors is more restricted at boundaries. Equation ( 2 ) describes the dynamics of the HAM mRNA. k hrp is the parameter for HAM mRNA production. Here we assumed that k hrp is constant in all cells within the SAM. This assumption is consistent with the experimental result that pHAM2::H2B-GFP reporter marker is highly expressed in all the layers of the SAM, including epidermis, sub-epidermis, and corpus. For degradation of HAM mRNA, we introduced both miR171 independent and dependent down-regulation terms. k hrnh is the parameter for the miR171 independent HAM mRNA degradation. We assumed that HAM mRNA degradation is further directly activated by local miR171, and this model assumption is supported by previous work [11] , [12] , [13] and our current work. k hrnm is the parameter for the miR171 dependent HAM mRNA degradation. Equation ( 3 ) describes dynamics of HAM protein. k hpp is the parameter for HAM protein production from HAM mRNA. k hpn is the parameter for HAM protein degradation. Equation ( 4 ) describes dynamics of H2B-GFP mRNA. k grp is the parameter for GFP mRNA production activated by ATML1 protein. k grn is the parameter for GFP mRNA degradation. Equation ( 5 ) describes dynamics of GFP protein. k gpp is the parameter for GFP protein production from GFP mRNA. k gpn is the parameter for GFP protein degradation. In the model, the functional ATML1 and PDF2 proteins in the SAM is set as an input ML1p, and levels of HAM mRNA and HAM protein are outputs. In the wild type SAM, ML1p is only present in the epidermal layer, so the [ML1p] is set as 1 a.u. in the epidermal layer cells and 0 a.u. in all the other cell layers of the SAM during the entire simulation time. When ATML1 is ectopically activated, one set of [ML1p] is defined based on the experimental results from the ATML1 RNA in situ hybridization in both wild type and the 35S::ATML1-GR plant (Supplementary Fig. 12 ). In the L1 of the 35S::ATML1-GR SAM, the level of ATML1 looks slightly higher than that in the wild type. Therefore, [ML1p] in the L1 of the 35S::ATML1-GR SAM was set to 1.1 a.u. At the deeper layers of the 35S::ATML1-GR SAM, the level of ATML1 is lower than that in the L1 layer of the same plant but higher than that in the deeper layers of the wild-type plant. Therefore, [ML1p] in deeper layers of the 35S::ATML1-GR SAM was set to 0.4 a.u. This set of [ML1p] is not based on quantitative analyses, due to the qualitative or at most semiquantitative nature of the RNA in situ hybridization method. The 1.1 a.u./0.4 a.u. in the ATML1 overexpression line vs 1 a.u./0 a.u. in the wild type in the model are qualitatively comparable to the patterns shown from the in situ result. To explore the effect of different [ML1p] values, a possible range of [ML1p] was assigned. Based on the RNA in situ images, the range is 1.05–1.5 a.u. for the L1 layer and 0.3–0.6 a.u. for the deep layers. Within this range, 24 different [ML1p] were randomly explored and used for the new simulations. Another possible set of [ML1p] values (1.3 a.u. in the L1 layer and 0.5 a.u. in deep layers) in this range is also included for the simulation. All these 25 sets of [ML1p] lead to suppressed HAM mRNA expression in deep layers of SAMs, which are largely comparable to the simulation result using the initial [ML1p] (1.1 a.u. in the L1 layer and 0.4 a.u. in deep layers), suggesting a robust response in the model when ATML1 protein is ectopically activated (Supplementary Movie 14 ). In addition to the [ML1p] patterns (Supplementary Movie 14 ) indicated by the RNA in situ images, other possible [ML1p] patterns were explored, to examine whether differences between [ML1p] in L1 and that in deep layers are important for HAM mRNA expression when ATML1 is ectopically activated in SAMs. In summary, new simulations were carried out using 50 sets of [ML1p] from a different range of values: 1.05-1.5 a.u. for the L1 layer and 0.6-2 a.u. for the deep layers (Supplementary Movie 15 ). Within this range, 24 different sets of [ML1p] were randomly identified and used for the new simulations. Another possible set of [ML1p] (1.1 a.u. in the L1 layer and 0.7 a.u. in deep layers) in this range is also included for the simulation (Supplementary Movie 15 ). Moreover, 24 additional sets of [ML1p] with the identical values for all SAM layers were randomly explored in the range of 1.05–1.5 a.u. and used for the simulations (Supplementary Movie 15 ). One set of [ML1p] (with 1.1 a.u. in all layers of SAM) is also included for the simulation. 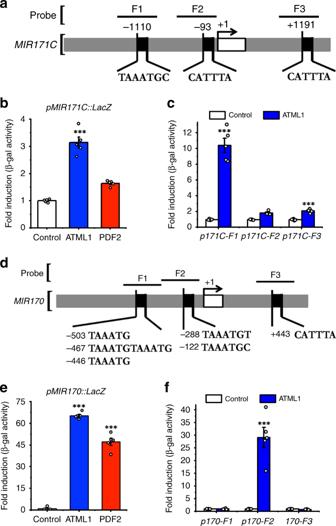Fig. 4: ATML1 binds to the promoters ofMIR171CandMIR170. aSchematic structure of theMIR171Cpromoter. The expanded diagram shows the sequences of putative L1 boxes on the promoter. Probes indicate the DNA fragments used in the Y1H assay. +1 indicates the transcription start site.bThe full-length promoter ofMIR171Cinteracts with ATML1 protein in Y1H. Y-axis: the relative activity of thepMIR171C::lacZ. All the numbers are normalized to the average value of the empty vector control. Bars: mean ± SE (n= 5 biological replicates). ***P< 0.001 (Student’s two-tailedt-test).cTheMIR171C-F1fragment from theMIR171Cpromote interacts with the ATML1 protein in Y1H. Y-axis: the relative activity of thepMIR171C-F1::lacZ,pMIR171C-F2::lacZandpMIR171C-F3::lacZreporters. All the numbers are normalized to the average value of the empty vector control. Bars: mean ± SE (n= 5 biological replicates). ***P< 0.001 (Student’s two-tailedt-test).dSchematic structure of theMIR170promoter. The expanded diagram shows the sequences of putative L1 boxes on the promoter. Probes indicate the DNA fragments used in the Y1H assay. +1 indicates the transcription start site.eThe full-length promoter ofMIR170interacts with ATML1 protein in Y1H. Y axis: the relative activity of thepMIR170::lacZreporter. All the numbers are normalized to the average value of the empty vector control. Bars: mean ± SE (n= 5 biological replicates). ***P< 0.001 (Student’s two-tailedt-test).fTheMIR170-F2fragment from theMIR170promoter interacts with the ATML1 protein in Y1H. Y-axis: the relative activity of eachlacZreporter. All the numbers are normalized to the average value of the empty vector control. Bars: mean ± SE (n= 5 biological replicates). ***P< 0.001 (Student’s two-tailedt-test). Source data underlying Fig.4b, cand Fig.4e, fare provided as a Source Data file. All these 50 new sets of [ML1p] lead to suppressed simulated HAM mRNA expression in deep layers of SAMs (Supplementary Movie 15 ), which are largely comparable to the simulation result using the initial [ML1p] (1.1 a.u. in the L1 layer and 0.4 a.u. in deep layers), suggesting the repression of HAM mRNA expression in the SAM when ATML1 is ectopically activated is not sensitive to differences between [ML1p] in L1 and that in deep layers. Note that in simulations that compare the SAMs from wild-type plants and plants with ectopic activation of ATML1, the only difference was the [ML1p], and all the parameters (shown in Supplementary Table 1 ) were the same. All simulations were carried out using the explicit forward Euler method with fine fixed time steps (0.01 h). At initial time point ( t = 0 h), all five dynamic agents (miR171, HAM mRNA, HAM protein, H2B-GFP mRNA from MIR171 transcriptional reporter, H2B-GFP protein from MIR171 transcriptional reporter) were set as 0 a.u. All simulations were carried out from initial time point to steady stages. To visualize the gene expression patterns in deeper layers in the simulation results, only half of the simulated SAM was shown in figures. In the five differential equations in the model, Eqs. ( 1 ) and ( 2 ) are the two equations that determine the dynamics of miR171 and HAM mRNA expression patterns, which are central components of our model. Equation ( 3 ) simply describes the universal relation between HAM protein and HAM mRNA, which does not provide novel property for HAM gene expression pattern. Equations ( 4 ) and ( 5 ) describe the dynamics of the H2B-GFP mRNA and H2B-GFP protein of the MIR171 transcriptional reporter reflecting the regulation of the MIR171 promoter, which do not feedback regulate miR171 or HAM mRNA levels, thus not essential for understanding the behavior of model in terms of miR171 and HAM mRNA pattern formation. Due to the above-mentioned reasons, the six parameters involved in Eqs. ( 1 ) and ( 2 ) were the focus for further exploration and analysis. The selected parameter values ranging from 40 to 200% of the initial value (Supplementary Table 1 ) were explored and sampled at 2% intervals. In total, from simulated results using 481 sets of parameters, 235 sets of parameters can lead to the apical-basal patterns of HAM mRNA in the SAM qualitatively comparable to experimental observations. See Supplementary Table 2 and Supplementary Data 1 for the ranges and values of these parameters. In addition to the local search based on the initial set of parameters (Supplementary Table 2 , Supplementary Data 1 ), an unbiased random search was performed using quasi Monte Carlo method. In summary, a total of 173 new sets of different parameters were identified (Supplementary Data 3 ) from 20,000 sets of random parameters (Supplementary Data 2 ). Simulation using each of the 173 parameter sets is able to qualitatively represent the HAM mRNA pattern experimentally observed in the wild type SAM (Supplementary Movie 13 ). Details of the random search are listed below. First, the low and high limit of each parameter was defined for the random search, based on knowledge of biological context in general and specific features of the regulatory system in the SAM being studied. Because a wild type SAM is dynamically stable, the production and degradation of the same agent (RNA/protein) need to be balanced. Therefore, the production and degradation rates for the agent were set to vary within a 100-fold range. In addition, because the miR171 regulates the HAM mRNA levels through direct binding and cleavage, the difference of turnover rates for these two agents is set within a 100-fold range. With these considerations, the search for parameter values was performed in the range of 0.1-1 for miR171 production rate, miR171 degradation rate, HAM mRNA production rate, miR171 dependent HAM mRNA degradation rate, and miR171 independent HAM mRNA degradation rate (the unit for each parameter is listed in Supplementary Table 1 ). Further, because movement of microRNAs between cells in the SAM is generally limited [33] , the search for parameter values of miR171 rescaled diffusion constant (rescaled by cell size) was defined in the range of 0.001–0.1 (area a.u./h). Within the defined ranges, Quasi Monte Carlo Method was used to randomly sample 20,000 sets of six different parameters uniformly on the log-scale (Supplementary Data 2 ). Then, simulations were performed using each of these 20,000 random parameter sets in the 3D template to search for more solutions for HAM mRNA patterns in the SAM. After comparing these simulation results (Supplementary Movie 13 ), 173 new sets of solutions (shown in Supplementary Data 3 ) were identified, which are different from the initial set of parameters (shown in Supplementary Table 1 ). The sensitivity of the total HAM mRNA (model output) to variations of six key parameters was analyzed [47] . Specifically, the parameters are increased by 1%. The sensitivity is computed as: \(\frac{{\Delta m}}{{\Delta p}} \times \frac{p}{m}\) . p is the original parameter value. Δp is the variation of the parameter. m is the total HAM mRNA expression. Δm is the variation of the total HAM mRNA expression. This sensitivity of all 6 key parameters is computed using 235 sets of parameter values (Supplementary Fig. 10 ) or 173 sets of parameters defined by the random search (Supplementary Fig. 11 ). In general, the model output shows robust behavior to variations of the six parameters. The total level of HAM mRNA shows higher degree of sensitivity to three parameters, including HAM mRNA production rate ( k hrp ) and miR171 independent HAM mRNA degradation rate ( k hrnh ), which directly control the production and degradation of HAM mRNA, respectively, and ( k mirn ), which determines the degradation of miR171. RT-qPCR The levels of gene expression in both Mock-treated and Dex-treated 35S::ATML1-GR plants were quantified through the real-time RT-PCR. 35S::ATML1-GR plants lines 5 and 9 were grown in short days for 20 days. 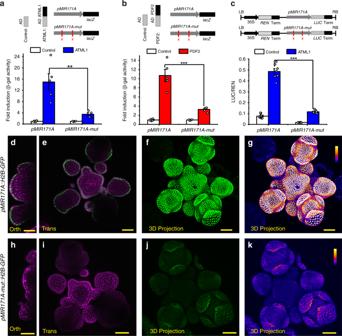Fig. 5: Epidermis specific cis-regulatory elements are required for the activation of miR171. a,bMutations in theMIR171Apromoter significantly reduced its interaction with ATML1 (a) or PDF2 (b) in Y1H. Upper panel: sketch of the reporter used in the study. AD with no fusion protein was included as the control. ThelacZreporter was under the control of either theMIR171Apromoter (pMIR171A::lacZ) or theMIR171Apromoter with two sites of TTAAATGC mutated (pMIR171A-mut::lacZ). Lower panel: mutations inpMIR171Asignificantly reduced the activation of thepMIR171A::lacZby ATML1 (a) or PDF2 (b). Bar: mean ± SE (a:n= 5 biological replicates for AD control and AD-ATML1, except thatn=4biological replicates for AD-ATML1 onpMIR171A-mut::lacZ;b:n= 5 biological replicates for AD control and AD-PDF2). **P< 0.01, ***P< 0.001 (Student’s two-tailedt-test).cDual-luciferase assay shows that the activation ofMIR171Apromoter activities by ATML1 is greatly compromised by the two mutations in theMIR171Apromoter. The LUC/REN in cells co-transformed with thepMIR171A::LUCreporter and the ATML1 effector (n= 7 biological replicates) is significantly higher than that in tobacco cells co-transformed with thepMIR171A-mut::LUCreporter and the same effector (n= 8 biological replicates). ***P< 0.001 (Student’s two-tailedt-test).d–gExpression ofpMIR171A::H2B-GFPin anArabidopsisSAM, from the orthogonal view (d), in the transverse optical section in corpus (e), and from the 3D projection view (f,g).h–kExpression ofpMIR171A-mut::H2B-GFPin the SAM, from the orthogonal view (h), transverse optical section view in corpus (i), and from the 3D projection view (j,k). The confocal settings for imaging GFP ind–kare identical, and the quantification of GFP is indicated by the identical color bar ing,k.d,e,h,i: merge of GFP (green) and PI counterstain (purple);f,j: GFP (green);g,k: GFP quantified fromf,j(quantification indicated by color). Scale bar: 20 µm; color bar ing,k: fire quantification of the signal intensity. Source data underlying Fig.5a–care provided as a Source Data file. After that, they were sprayed with mock (no Dex) or with 10 µM DEX solution. After 24 h, the whole shoots were cut off from the top of hypocotyls and harvested for RNA extraction and RNA was isolated using RNeasy Mini Kit (Qiagen). Reverse transcription was performed from 1.2 µg total RNA using SuperScript Reverse Transcriptase (ThermoFisher). Quantitative PCR was performed using SYBR Green qPCR Master Mix (Bimake) on a BioRad CFX96. The primers for UBC (as the internal control) qPCR are described previously [7] . The primers for GFP are 5′-GAACCGCATCGAGCTGAA-3′ and 5′-TGCTTGTCGGCCATGATATAG-3′. The primers for MIR171A : 5′-GATATTGGCCTGGTTCACTC-3′ and 5′-CCACAAAGTCCAAAATAGAG-3′ and for MIR171B : 5′-GGAGCTAAGTGGAGATTATAG-3′ and 5′-GGTTATAATAACTATCTTTGCC-3′ as described previously [13] . The primers of HAM1 and HAM2 qPCR were designed to span their miR171 targeting sites. For HAM1 : 5′-AAACAACAACGGCGACCA-3′ and 5′-CTTTGAAACGGAGACTTGTGG-3′ were used. For HAM2 : 5′-CAAACGGCGGAGATAACAAT-3′ and 5′-CTGTGGAACGGAGGTTTAGG-3′ were used. The mean and standard error was calculated from three independent biological replicates. 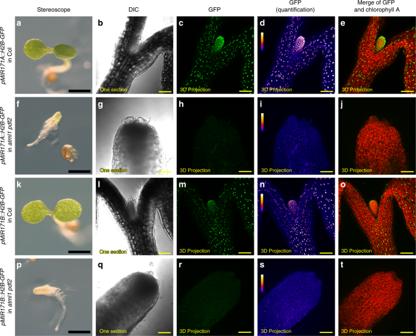Fig. 6: Epidermal specification pathway is required for the expression ofMIR171genes. a–eThe wild type seedling (Col) expressing thepMIR171A::H2B-GFPreporter.f–jTheatml1 pdf2double mutant seedling expressing thepMIR171A::H2B-GFPreporter.k–oThe wild type seedling (Col) expressing thepMIR171B::H2B-GFPreporter.p–tTheatml1 pdf2double mutant expressing thepMIR171B::H2B-GFPreporter. Panels (from left to right): seedlings used for the confocal imaging; DIC from one optical section; GFP (green) in 3D projection view, quantified GFP (quantification indicated by color) in 3D projection view; merge of GFP (green) and chlorophyll (red) in 3D projection view. Scale bars: 1 mm (a,f,k,p) and 100 µm (b–e,g–j,l–o, andq–t); color bar (d,i,n,s): fire quantification of the signal intensity. 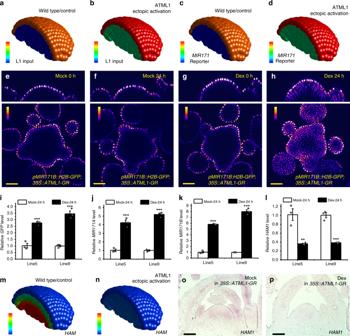Fig. 7: The 3D computational model simulates the L1-miR171-HAM regulatory circuit in SAMs. a,bInput of the ATML1 level (L1 input) for the computational simulation in (c,m) and (d,n). Color indicates the level of ATML1 input, with the gradient from red (maximum, 1.1 a.u.) to blue (none).c,dSimulated promoter activity ofMIR171in the SAMs from the wild type control (c) and the plant with ectopic activation of ATML1 (d). Color indicates the simulatedMIR171reporter activity, with the gradient from red (maximum, 1.1 a.u.) to blue (none).e–hConfocal live imaging of thepMIR171B::H2B-GFPreporter in the SAMs of35S::ATML1-GRplants, with the mock control (e,f) and the Dex treatment (g,h). Using identical imaging settings, the same SAM was imaged at 0 h and 24 h after the indicated treatment. Colors indicate quantified GFP intensities, and color bars represent fire quantification of signal intensity. Panels: (top) orthogonal view; (bottom) transverse optical section view from corpus.i–lQuantification of the gene expression forGFP(i),MIR171A(j),MIR171B(k), andHAM1(l) in two independent35S::ATML1-GR; pMIR171B::H2B-GFPtransgenic lines (#5 and #9) 24 h after the mock or Dex treatment. Bars: mean ± SE. **P< 0.01, ***P< 0.001 (Student’s two-tailedt-test).n= 3 biological replicates.m,nSimulatedHAM1mRNA expression patterns in SAMs from the wild type control (m) and the plant with ectopic activation of ATML1(n). Color indicates the simulatedHAM1mRNA levels, with the gradient from red (at or above 2 a.u.) to blue (none).o,pRNA in situ hybridizations forHAM1mRNA in the SAMs of35S::ATML1-GR;pMIR171B::H2B-GFPplants 5 days after the mock (o) or Dex (p) treatment. One set of representative results are shown, and similar results from three independent biological replicates were obtained for each treatment. Scale bar: 50 µm (o–p). The template of a whole SAM was used for all the simulations, and only a half of the SAM is displayed for visualization of cells in inner layers. Source data underlying Fig.7i–lare provided as a Source Data file. 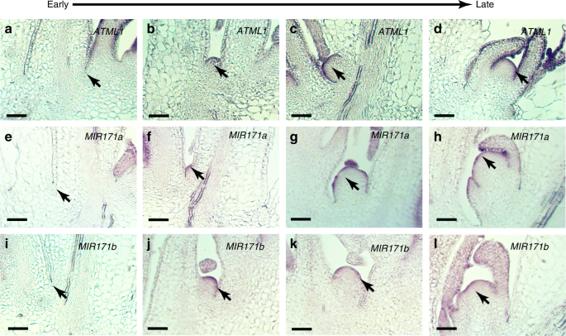Fig. 8: Pattern formation of L1 and miR171 in de novo axillary stem cell niches. a–dRNA in situ hybridization ofATML1mRNA in wild-type (Ler) plants, from early to late developmental stages during the de novo formation of the axillary meristem (AM).e–hRNA in situ hybridization ofGFPmRNA inpMIR171A::H2B-GFPplants showing the promoter activity ofMIR171A, from early to late stages of AM initiation.i–lRNA in situ hybridization ofGFPmRNA inpMIR171B::H2B-GFPplants showing the promoter activity ofMIR171B, from early to late stages of AM initiation. The results have been confirmed by three biological replicates. Scale bar: 50 µm. Reporting summary Further information on research design is available in the Nature Research Reporting Summary linked to this article.